Blocking Dectin-1 prevents colorectal tumorigenesis by suppressing prostaglandin E2 production in myeloid-derived suppressor cells and enhancing IL-22 binding protein expression Dectin-1 (gene Clec7a ), a receptor for β-glucans, plays important roles in the host defense against fungi and immune homeostasis of the intestine. Although this molecule is also suggested to be involved in the regulation of tumorigenesis, the role in intestinal tumor development remains to be elucidated. In this study, we find that azoxymethane-dextran-sodium-sulfate-induced and Apc Min -induced intestinal tumorigenesis are suppressed in Clec7a −/− mice independently from commensal microbiota. Dectin-1 is preferentially expressed on myeloid-derived suppressor cells (MDSCs). In the Clec7a −/− mouse colon, the proportion of MDSCs and MDSC-derived prostaglandin E 2 (PGE 2 ) levels are reduced, while the expression of IL-22 binding protein (IL-22BP; gene Il22ra2 ) is upregulated. Dectin-1 signaling induces PGE 2 -synthesizing enzymes and PGE 2 suppresses Il22ra2 expression in vitro and in vivo. Administration of short chain β-glucan laminarin, an antagonist of Dectin-1, suppresses the development of mouse colorectal tumors. Furthermore, in patients with colorectal cancer (CRC), the expression of CLEC7A is also observed in MDSCs and correlated with the death rate and tumor severity. Dectin-1 signaling upregulates PGE 2 -synthesizing enzyme expression and PGE 2 suppresses IL22RA2 expression in human CRC-infiltrating cells. These observations indicate a role of the Dectin-1-PGE 2 -IL-22BP axis in regulating intestinal tumorigenesis, suggesting Dectin-1 as a potential target for CRC therapy. Colorectal cancer (CRC) is the third most common type of cancer in the world, with over 1 million new cases and 500,000 deaths globally every year [1] . Most CRC cases occur in old age and dietary habit is suggested to be a possible risk factor for CRC [2] . However, underlying mechanisms that regulate intestinal tumor development have not been elucidated completely. The C-type lectin receptor (CLR) is a family molecules consisted of more than 100 proteins with one or more lectin-like carbohydrate-recognition domains, which recognize a broad repertoire of ligands in the extracellular domain and a signal transducing motif, such as immunoreceptor tyrosine-based activation motif (ITAM) and immunoreceptor tyrosine-based inhibitory motif (ITIM), in the intracellular domain and regulate a diverse range of immunological functions [3] . Dectin-1 (gene symbol: Clec7a ), one of CLRs preferentially expressed in myeloid-derived cells, is the receptor for β−1, 3-linked glucans (β-glucans) [4] , [5] , [6] . Since β-glucans are the major cell wall components of most fungi, Dectin-1 stands on the first line of the host defense against fungal infection [5] , [6] . Furthermore, recent studies have revealed that this receptor is also involved in the development of allergic, autoimmune, and cancerous diseases [3] , [7] . Dectin-1 signaling is reported to aggravates airway hypersensitivity by inducing proallergic chemokines and mucus [8] , and administration of a Dectin-1 agonistic ligand curdlan evokes arthritis, spondyloarthritis and ileitis in an autoimmune-prone mouse with a spontaneous mutation in ZAP-70 [9] , [10] . Recently, we reported that Dectin-1-deficiency causes overexpansion of a commensal bacterium Lactobacillus murinus , which induces regulatory T (Treg) cell differentiation, in the mouse colon, resulting in the suppression of dextran sodium-sulfate (DSS)-induced colitis [11] . Dectin-1 signaling also induces IL-17F in the downstream and suppresses the growth of a group of commensal bacteria including Clostridium cluster XIVa, which also promotes Treg differentiation, by inducing specific antimicrobial proteins [12] , [13] . Therefore, although Dectin-1 basically activates the immune system to eradicate pathogens, this activity, on the other hand, can also trigger or enhance inflammation-related diseases. A large number of studies were carried out about the effects of β-glucans and Dectin-1 signaling on the development of tumors, especially because we are taking lots of β-glucans as a component of daily foods such as yeasts, mushrooms, and seaweeds, and also as a herbal medicine [14] , [15] . However, these results are sometimes contradictory each other. Many reports suggest a protective role for Dectin-1 signaling in the development to tumors. Oral administration of high molecular weight (MW) β‐glucans suppresses the growth of subcutaneously inoculated Lewis lung carcinoma [16] . Orally administrated β-glucans also enhance the effects of antibody therapy through modification of antitumor immunity [17] , [18] . Furthermore, β-glucan injection prevents mouse liver metastases of transferred C-26 colon carcinoma cells [19] . Although some studies suggest direct tumor cell growth inhibitory activity of β-glucans, it is now recognized that β-glucans have no such cytotoxic effects [20] , [21] . Dectin-1 signaling was reported to enhance tumor-killing activity of NK cells through induction of INAM on DCs by binding N-glycans on B16 melanoma cells [22] . Dectin-1 upregulates TNFSF15 and OX40L expression in DCs to promote anti-tumorigenic Th9 cell differentiation by activating Raf1 and NF-κB [23] . Dectin-1 also suppresses chemical carcinogen-induced hepatocellular carcinogenesis by suppressing Toll-like receptor (TLR) 4-dependent inflammation [24] . In contrast, a tumor promotive role for the Dectin-1 signaling was reported in pancreatic tumorigenesis. In that report, Dectin-1 recognizes non-canonical endogenous ligand galectin-9 expressed on pancreatic ductal adenocarcinoma to suppress anti-tumorigenic M1 macrophage differentiation [25] . However, until now, no study has elucidated the function of Dectin-1 in the development of intestinal tumors. In this study, we investigate the role of Dectin-1 in colorectal tumorigenesis by analyzing mouse intestinal tumor models and CRC patients. We show that Dectin-1 signaling rather promotes the development of colorectal tumors by enhancing the production of prostaglandin E2 (PGE 2 ), which facilitates CRC development and suppresses the expression of tumor-inhibitory IL-22-binding protein (IL-22BP). These observations reveal a tumor promotion pathway in the intestinal tract and suggest Dectin-1 as a possible target for the therapy of CRC. Dectin-1-deficiency suppresses colorectal tumor development in a commensal microbiota-independent manner To investigate the potential role of Dectin-1 in intestinal tumorigenesis, we first examined the influence of Clec7a gene deficiency ( Clec7a −/− ) on the development of colorectal tumor in DSS-treated Apc Min ( Apc Min -DSS) mice, in which intestinal adenoma is induced due to enhanced β-catenin activity [26] . Body weight loss in Apc Min/+ Clec7a −/− mice after DSS-treatment was significantly milder than that in Apc Min/+ mice (Fig. 1a ), and at day 28 after DSS-treatment, polyp number in the colon was significantly reduced in Apc Min/+ Clec7a −/− mice (Fig. 1 b, c ). Shortening of colon length, one of the symptoms of colitis, was milder in Apc Min/+ Clec7a −/− mice (Fig. 1 c, d ), as observed in DSS-treated Clec7a −/− mice [11] . Fig. 1: Dectin-1-deficiency suppresses development of colorectal tumors without involvement of commensal microbiota. a – f Apc Min/+ and Apc Min/+ Clec7a −/− mice at 8–10 weeks old were treated with 1% DSS for 7 days and were sacrificed 4 weeks later. Body weight changes were observed chronologically after DSS-treatment ( a , day5, ** P = 0.0098; day9, * P = 0.0297; day10, * P = 0.0127, day12, * P = 0.0260; day14, * P = 0.0364). Number of colorectal polyps with indicated size ( b , <2 mm, * P = 0.0130; >3 mm, ** P = 0.00139; Total, ** P = 0.00948), representative gross pathology of the colon ( c ) and colon length ( d , *** P = 0.00018) are shown ( n = 5/group). Representative H.E.-stained histology of the polyps ( e ) and histopathological scores ( f , Apc Min/+ n = 7, Apc Min/+ Clec7a −/− n = 5; *P = 0.0152) are shown. g – l WT and Clec7a −/− mice were i.p. administrated with AOM, and 7 days later, they were treated with 1% DSS for 3 cycles (AOM-3DSS) as described in Methods. Body weight loss was inspected chronologically during the induction of colorectal tumor ( g , day15, * P = 0.0352; day32, ** P = 0.00129; day35, * P = 0.0237; day36, ** P = 0.0088; day37, * P = 0.0338; day46, * P = 0.0475; day52, * P = 0.0339; day53, * P = 0.0179; day57, * P = 0.0290; day58, * P = 0.0276; day59, * P = 0.0119; day60, * P = 0.0251; day61, * P = 0.0196). Mice were sacrificed at week 16 after AOM administration, and number of colorectal polyps with indicated size ( h , 2–3 mm, * P = 0.0150; >3 mm, * P = 0.0339; Total, * P = 0.0312), gross pathology of the colon ( i ), colon length ( j , * P = 0.0103), representative histology of the polyps ( k ) and histopathological scores ( l , * P = 0.0159, ** P = 0.0079) are shown ( n = 5/group). m – o GF WT and Clec7a −/− mice were treated with AOM-3DSS. Thirty-six weeks after AOM administration, these mice were sacrificed, and gross pathology of the colon ( m ) and colon length ( o ) are shown. Colorectal tumor sizes in indicated mice were measured and total polyp volume ( n , **** P < 0.0001) is shown. The polyp volume was calculated as (diameter) 3 for circular polyps and as (Short diameter) 2 × (long diameter) for elliptic polyps (n = 4/GF WT group, n = 5/GF Clec7a −/− group). Data in (a-f) are representatives of five, in g – l are representatives of six, and in m - o are representatives of three independent experiments. Data in a , b , d , f , g , h , j , l , n , o are presented as means ± SD. Data in a , b , d , g , h , j , n , o are analyzed using unpaired two-tailed Student’s t -test and in f , l using two-tailed Mann–Whitney U -test. Source data are provided in the Source Data file. Full size image We also examined the effect of Dectin-1-deficiency on spontaneous tumor development in Apc Min mice. After sacrificing mice at 20–23 weeks of age, we found the number of polyps in both small and large intestines was significantly decreased in Apc Min/+ Clec7a −/− mice compared with that in Apc Min/+ mice (Supplementary Fig. 1a – d ). Histologically, complex budding of crypts and high- or low-grade dysplasia or hyperplasia in both colon and rectum were observed in Apc Min/+ mice, while these histopathological changes were reduced in Apc Min/+ Clec7a −/− mice (Fig. 1 e, f ). We further analyzed a chemically induced colorectal tumor model in which mice were treated with azoxymethane (AOM), followed by 3 cycles of DSS treatment (AOM-3DSS). Clec7a −/− mice exhibited milder body weight loss than wild-type (WT) mice during 3 cycles of DSS-treatment (Fig. 1g ), and the polyp number in Clec7a −/− mice was significantly smaller than that in WT mice (Fig. 1 h, i ). Shortening of the colon length was significantly milder in Clec7a −/− mice (Fig. 1 i, j ). When mice were treated with AOM and only one cycle of DSS, anal prolapse (Supplementary Fig. 1e , f ) and shortening of colon length (Supplementary Fig. 1g, h ) were also significantly milder in Clec7a −/− mice. Although all the WT mice developed colorectal polyps, only half of Clec7a −/− mice developed polyps with smaller sizes (Supplementary Fig. 1f, i ). Histologically, complex budding of crypts, high-grade dysplasia or hyperplasia were only observed in both colon and rectum section of WT mice, and only mild levels of the lesions and crypt changes were observed in those of Clec7a −/− mice (Fig. 1 k, l ). Submucosal invasion was not observed in these AOM-DSS-treated mice. All these results indicate that blockade of Dectin-1 signaling inhibits intestinal tumorigenesis. We previously reported that DSS-induced colitis is suppressed in Clec7a –/– mice, because colonization of a regulatory T cell (Treg)-inducing commensal bacterium Lactobacillus murinus is increased in the intestine of Clec7a −/− mice [11] . Actually, real-time RT-PCR and flow-cytometry analysis showed that Foxp3 (Treg marker) expression and Foxp3 + CD4 + T cell proportion in polyps and non-polyp tissue were significantly increased in Dectin-1-deficient mice (Supplementary Fig. 1r , t ). To examine the effects of intestinal microbiota in the regulation of tumorigenesis in Clec7a −/− mice, we continuously co-housed Clec7a −/− mice with WT mice after weaning to harmonize intestinal microbiota and treated them with AOM-3DSS. Body weight loss and shortening of colon length caused by DSS-treatment were similar between these co-housed mice (Supplementary Fig. 1j, l, m ), but the polyp number of colon and rectum in Clec7a −/− mice was still significantly fewer than those in WT mice (Supplementary Fig. 1n ), especially of larger sizes (diameter >3 mm, Supplementary Fig. 1k, l ), as that seen in separately housed mice. We next examined the involvement of commensal microbiota in the effect of Dectin-1-deficiency on intestinal tumorigenesis in Apc Min -DSS model. Apc Min/+ and Apc Min/+ Clec7a −/− mice were pretreated with antibiotics (ABX) for 3 weeks, then DSS + ABX were administered for 1-week, followed by continuous ABX-treatment for another 4 weeks. Apc Min/+ Clec7a −/− mice developed less number of polyps compared with Apc Min/+ mice, although total polyp number was decreased in ABX-treated mice (Supplementary Fig. 1o – 1q ). To further exclude the effects of commensal microbiota on Dectin-1-mediated colorectal tumor regulation, we generated germ-free (GF) mice and treated them with AOM-3DSS. Thirty-six weeks after AOM administration, we observed that colorectal polyps were developed only in WT but not in Clec7a −/− GF mice (Fig. 1 m, n ), although the colon length of these mice was similar (Fig. 1 m, o ). Intestinal Foxp3 expression was similar between WT and Clec7a −/− GF mice (Supplementary Fig. 1s ), indicating the Treg population is similar. We also found the expression of Ccnd1 encoding Cyclin-D1, which promotes cell cycle progression, was downregulated in Clec7a −/− mice under both SPF and GF conditions (Supplementary Fig. 1r, s ), consistent with the suppression of tumor growth in Clec7a −/− mice. These results indicate that commensal microbiota are not involved in the suppression of tumorigenesis in Clec7a −/− mice. Infiltration of myeloid-derived suppressor cells (MDSCs) is decreased in polyps in Clec7a −/− mice To elucidate the mechanism by which Dectin-1-deficiency suppresses intestinal tumorigenesis, we examined Dectin-1 expressing cells in tumors of Apc Min -DSS mice. Flow cytometric analysis showed that Dectin-1 was mainly expressed on CD103 – CD11c – CD11b + cells in colonic polyps (Fig. 2a , 92.4%). Nearly 75% of these Dectin-1 + cells were MHC-II – cells, in which approximately 50% were Ly6C int Ly6G + CD11b + , 5% were Ly6C hi CD11b + and 19% were MHC-II – Gr1 – CD11c – CD11b + cells (Supplementary Fig. 2a ). These tumor-infiltrating Ly6C int Ly6G + CD11b + and Ly6C hi CD11b + myeloid cells are commonly known as granulocytic polymorphonuclear- (PMN-) and monocytic- (M-) MDSCs [27] , respectively. Fig. 2: MHC-II + CD11c – CD11b + cell population is decreased in the colon of Clec7a –/– mice. a Apc Min/+ and Apc Min/+ Clec7a −/− mice were treated with 1% DSS for 7 days and were sacrificed 4 weeks later. Flow cytometric analysis was carried out to identify Dectin-1-expressing cells in colorectal polyps and non-polyp tissues. b , c Apc Min/+ and Apc Min/+ Clec7a −/− mice were treated with 1% DSS for 7 days and were sacrificed 4 weeks later. Proportions of T cells, B cells and DCs in total tissue-infiltrating cells ( b , αβT cells, ** P = 0.0020; γδT cells, ** P = 0.0076; CD19 + B cells, ** P = 0.0069; IgG + B cells, ** P = 0.0058; CD11c + DCs, ** P = 0.0014, **** P < 0.0001), and proportions of MHC-II + CD11c + and MHC-II + CD11c – CD11b + cells in tissue-infiltrating CD45 + cells ( c , MHC-II + CD11c + , ** P = 0.0039, * P = 0.0157; MHC-II − CD11c − CD11b + , * P = 0.0563, **** P < 0.0001) in non-polyp tissues or polyps in the colon were examined by flow cytometry ( n = 3/ Apc Min/+ group, n = 5/ Apc Min/+ Clec7a −/− group). d WT mice were treated with AOM-3DSS and were sacrificed after 12 weeks. Indicated types of cells in polyps and non-polyp tissues were purified with autoMACS and Il6 and Il1b expression was examined by RT-qPCR ( n = 3 biologically independent samples/group). e WT mice were administrated with AOM followed by 3 cycles of DSS. After 11 weeks of AOM treatment, these mice were sacrificed and CD11b + and CD11c + cells were purified from colorectal polyps with autoMACS. The sorted cells were stimulated with an agonistic β-glucan OXCA for 16 h with or without pretreatment with an antagonistic β-glucan laminarin, for 3 h, then, Il6 and Il1b expression were determined by RT-qPCR ( n = 4 biologically independent samples/group; in Il6 panel, *** P = 0.0002, * P = 0.0382; Il1b panel, **** P < 0.0001, ** P = 0.0012). Data in a – e are representatives of two independent experiments. Data in b – e are expressed as means ± SD. Data in b , c are analyzed using two-way analysis of variance (ANOVA) and in e using one-way ANOVA followed by Tukey’s multiple-comparisons test. Source data are provided in the Source Data file. Full size image We next analyzed tumor-infiltrating cell populations in the colon, and found that infiltration of T cells (including αβ & γδ T cells), B cells (including IgG + B cells), and DCs (MHC-II + CD11c + cells) was significantly increased in Apc Min/+ Clec7a −/− mice (Fig. 2b ; Supplementary Fig. 2 b, c ), suggesting enhanced immune responses in Apc Min/+ Clec7a −/− mice compared with Apc Min/+ mice. In contrast, MHC-II – CD11c – CD11b + population was decreased in polyps of these Clec7a −/− mice (Fig. 2c ; Supplementary Fig. 2c ). We further showed that both CD11c – CD11b + Ly6C int and CD11c – CD11b + Ly6C hi population were reduced in the polyps of Apc Min/+ Clec7a −/− mice (Supplementary Fig. 2d ), suggesting that Dectin-1 signaling facilitates MDSC expansion in intestinal tumors. IL-6 and IL-1β are reported to promote MDSC expansion [28] , [29] . When we purified EpCAM + epithelial cells, CD11b + and CD11c + myeloid cells, Thy1.2 + T cells, CD19 + B cells and other CD45 + leukocytes from intestinal polyps and non-polyp tissues, we found that Il6 mRNA was expressed by both myeloid cells and T cells, and Il1b was exclusively detected in myeloid cells in both polyp and non-polyp tissues (Fig. 2d ). When these polyp-infiltrating CD11b + and CD11c + cells were stimulated with a β-glucan OXCA from Candida albicans , Il6 and Il1b mRNA expression and IL-6 and pro-IL-1β protein expression were induced, and this induction was inhibited by a Dectin-1 antagonist laminarin (Fig. 2e ; Supplementary Fig. 2e ). These results support the idea that MDSC expansion in WT mouse polyps is caused by Dectin-1 signaling-induced cytokine(s) at least in part. The expression of genes for PGE 2 synthesizing enzymes is decreased, while that for IL-22BP is increased in Clec7a −/− mice Next, we examined gene expression by RNA-seq analysis in colonic tumors and non-tumor tissues from AOM-3DSS-treated GF mice, as we could detect the difference between WT and Clec7a −/− mice more clearly than using SPF mice. This is probably because the influence of microbiota on gene expression was excluded in GF mice. The expression of genes associated with T cells ( Cd3e , Cd28 , Cd69 , Ccr6 , Ccr9 ), Th1 cells ( Cd4 , Tbx21 , Ifng , Il12a , Cxcr3 ), B cells ( Cd19 , Ig-associated, Cxcr5 ), and DCs ( Cd80 , Cd86 , Itgax , H2-Ab1 , Ccr7 ) was upregulated in polyps of Clec7a −/− mice (Fig. 3a ; Supplementary Fig. 3a , b ), consistent with the results in Fig. 2 b, c . The expression of cytokines such as Il1b, Il17a and Il23a , and chemokines such as Ccl1, Ccl2, and Cxcl2 was downregulated in polyps of Clec7a −/− mice (Fig. 3a ; Supplementary Fig. 3b ). Interestingly, the expression of IL-22-binding protein (IL-22BP; gene: Il22ra2 ), which is suggested to be involved in colorectal tumor regulation [30] , was upregulated in polyps of Clec7a −/− mice (Fig. 3a ; Supplementary Fig. 3a ). Fig. 3: The expression of genes encoding PGE 2 -synthesizing enzymes and IL-22BP is regulated by Dectin-1 signaling. a – d GF WT and Clec7a −/− mice treated with AOM-3DSS shown in Fig. 1m were sacrificed at 36 weeks after AOM administration, and RNA-seq analysis was carried out by using RNAs from polyps and non-polyp tissues in the vicinity (pooled 4 WT and 5 Clec7a −/− GF mice). Expression levels of genes for cytokine, chemokine, cell-surface marker, and T cell transcription factor in WT and Clec7a −/− mice are shown as heatmaps ( a ). Cell populations, signaling pathways and metabolic pathways were compared between Clec7a −/− and WT mouse polyps by using the KEGG database. Log2 (fold-change) > 1 is upregulated genes, while log2 (fold-change) <−1 is downregulated genes ( b ). Expression levels of MDSC-associated genes are presented as a heatmap ( c ). Expression levels of PGE 2 -synthase genes in polyp and non-polyp tissues are shown as a heatmap ( d ). e – h SPF WT and Clec7a −/− mice treated with AOM-3DSS for 16 weeks, and CD11b + and CD11c + cells were purified from colorectal polyps and were applied to scRNA-seq analysis. UMAP showing cell type cluster distribution ( e ), proportions of MDSC and DC subsets ( f ), changes of typical MDSC-associated gene expressions during MDSC development ( g ), and the trajectory tracks of the differentiation of PMN-MDSCs and M-MDSCs ( h ) in WT and Clec7a −/− mice are shown (5 WT and 4 Clec7a −/− mice pooled). i Bone marrow cells from WT mice were harvested and were stimulated with rGM-CSF and rIL-6 (2 × 10 5 cells/well) for 5 days. Curdlan with indicated doses was added on the 2nd day and flow cytometry was carried out to examine MDSC differentiation by staining with antibodies against Ly6C and CD11b. j After the culture in i , differentiated bone marrow cells were further co-cultured with splenic CD4 + T cells from WT mice for 2 days in the present of anti-CD3/CD28 microbeads. After the co-culture, proportions of CD11b + and CD4 + cells in CD45 + cells and the proportion of IFN-γ + cells in CD4 + cells were determined by flow cytometry ( n = 3 biologically independent samples/group; in CD11b + panel, *** P = 0.0009; in CD4 + T panel, **** P < 0.0001; in IFN-γ + panel, *** P = 0.0001). k EpCAM − MHC-II − Gr1 + cells were isolated from colonic polyps of AOM-3DSS-treated WT and Clec7a −/− mice and were co-cultured with splenic CD4 + T cells in the presence of anti-CD3/CD28 microbeads. Two days later, flow cytometry was carried out to determine the number of live CD4 + T cells (control n = 3, +WT MDSC n = 5, + Clec7a −/− MDSC n = 3, **** P < 0.0001). l Intestinal polyp-infiltrating cells were isolated from Apc Min/+ and Apc Min/+ Clec7a –/– mice, and proportions of NOS2-producing CD11c – CD11b + cells were determined by flow cytometry ( Apc Min/+ n = 6, Apc Min/+ Clec7a −/− n = 7, ** P = 0.0027). Data in i , j are representatives of three and in k is representative of two independent experiments. Data from two independent experiments are pooled in l and in j – l are expressed as means ± SD. Data in j , k are analyzed using one-way ANOVA followed by Tukey’s multiple-comparisons test and in l using unpaired two-tailed Student’s t -test. Source data are provided in the Source Data file. Full size image By KEGG gene enrichment analysis, we found that immune related genes such as antibody production, lymphocyte activation, NK cell-mediated cytotoxicity, and antigen presentation were upregulated in tumor tissues of Clec7a −/− mice compared to that of WT mice (Fig. 3b ). In contrast, pathways such as Wnt signaling, IL-17 signaling, Ras signaling, and arachidonic acid metabolism were downregulated in Clec7a −/− mouse colon (Fig. 3b ). The expression of characteristic genes of MDSC [31] , [32] was significantly decreased in Clec7a −/− mouse polyps (Fig. 3c ), consistent with decreased MDSC infiltration in colonic tumors in Clec7a −/− mice (Fig. 2c ). The expression of MDSC-differentiation-promotive cytokines, such as Csf2, Il6, Il1b and Tnf [28] , [29] , was decreased in Clec7a −/− mouse polyps (Fig. 3a ; Supplementary Fig. 3a , b ). Interestingly, we found that the expression of genes encoding prostaglandin E 2 (PGE 2 ) synthases, such as Pla2g2a / 2e (Phospholipase A2 group IIA/IIE), Ptgs1/2 (Cox1/Cox2), and Ptges2/3 (PGE 2 synthase 2/3), was downregulated in polyps in Clec7a −/− mice (Fig. 3d ; Supplementary Fig. 3a ). The expression of Clec7a was elevated in polyps compared with non-polyp tissues (Supplementary Fig. 3c ), reflecting the expansion of tumor-infiltrating MDSCs in which Dectin-1 was highly expressed. Then, we further analyzed gene expression in colonic polyp-infiltrating CD11b + and CD11c + cells from AOM-3DSS-treated mice by single-cell RNA-sequencing (scRNA-seq) analysis. Fifteen types (clusters) of myeloid cells were identified and they were further classified into four big groups; these are monocyte-associated (cluster #0, 1, 2), neutrophil-associated (#3, 8, 12), macrophage-associated (#5, 7, 10, 14) and DC-associated (#4, 6, 9, 11,13) (Fig. 3e ; Supplementary Fig. 3d ). Judging from the characteristic gene expression patten, cluster 2 was identified as M-MDSC and cluster 3 was PMN-MDSC. We found that both of these MDSC populations were decreased in Clec7a −/− mice compared with those in WT mice (Fig. 3 e, f ; Supplementary Fig. 3d ). In contrast, all the DC populations consisting of 5 subgroups were increased in Clec7a −/− mice compared with WT mice. Other myeloid-cell populations were not changed in Clec7a −/− mice (Supplementary Fig. 3e ). To further investigate the influence of Dectin-1 on the differentiation of each MDSC cell type, we carried out pseudo-time trajectory analysis by focusing on the monocyte group (cluster #0, 1, 2) and the neutrophil group (cluster #3, 8, 12). We found that the gene expression profiles between neutrophils and PMN-MDSC were closely related, and the expression levels of signature genes of MDSC, such as Arg2 , S100a9 and Csf3r , were gradually increased from neutrophil to PMN-MDSC (Fig. 3g ). Similar relationship was also observed between monocyte and M-MDSC (Fig. 3g ). During both types of MDSC differentiation, Il1b expression was also upregulated, but the average level of the mRNA as well as the protein in Clec7a −/− mice was lower than that in WT mice (Supplementary Fig. 3f, g ). By the trajectory analysis, PMN-MDSCs were shown to be differentiated from neutrophils through neutro.→ mdsc transitional state, in which typical MDSC gene Arg2 was not expressed yet (Fig. 3h ). We found that the differentiation of PMN-MDSCs was suppressed in Clec7a −/− mice (WT54.8% vs. KO10.8%) due to the blockade of the transition from neutro.→mdsc transitional cells to MDSCs, resulting in the accumulation of the transitional cells (KO66.3% vs. WT10.5%) (Fig. 3h ). Similarly, M-MDSC population was differentiated from monocytes through monocyte→M1 macrophage transitional cells, and this process was again suppressed in Clec7a −/− mice (KO17.0% vs. WT39.8%). Transition from monocyte→M1 macrophage transitional cells to M-MDSC was significantly suppressed in Clec7a −/− mice and accumulation of transitional cells were observed (KO63.6% vs. WT37.0%), although the frequency of monocytes was not much different between WT and Clec7a −/− mice (19.4% vs. 23.2%). These results suggest that Dectin-1 signaling plays important roles in the development of tumor-infiltrating MDSCs. To confirm the promotive role of Dectin-1 signaling in MDSC differentiation, we induced MDSC in vitro from bone marrow cells with GM-CSF and IL-6 [33] , and examined the effect of Dectin-1 agonistic ligand curdlan. As shown in Fig. 3 i, j , curdlan significantly enhanced Ly6C + CD11b + cell differentiation. The expression of genes typical for mouse MDSCs, such as Arg2 and Nos2 [32] , was upregulated by curdlan stimulation in a dose-dependent manner (Supplementary Fig. 3h ). When these cells were co-cultured with CD4 + T cells isolated from the spleen, these Dectin-1-induced myeloid cells suppressed anti-CD3/CD28-induced T cell proliferation and IFN-γ production in these cells (Fig. 3j ), indicating these cells represent MDSCs. When AOM-3DSS-induced colonic polyp-derived MHC-II − Gr1 + cells were co-cultured with splenic CD4 + T cells, T cell proliferation was suppressed by these tumor-infiltrating Gr1 + cells from WT mice, while Gr1 + cells from Clec7a −/− mouse polyps suppressed T cell population only weakly (Fig. 3k ). Co-culturing CD4 + T cells with Gr1 + cells isolated from the spleen of AOM-3DSS-treated mice also showed the similar impairment of immunosuppressive activity of Dectin-1-deficient Gr1 + cells (Supplementary Fig. 3i , j ). Drastic impairment of NOS2 secretion by intestinal polyp-infiltrating CD11c − CD11b + cells from Clec7a −/− mice is consistent with this T cell suppression (Fig. 3l ). All these observations indicate that Dectin-1 signaling facilitates both differentiation and immune-suppressive activity of intestinal MDSCs. Both T cells and B cells are suggested to be involved in antitumor immunity [34] , [35] , [36] , and both of them are increased in the intestinal polyps of Clec7a −/− mice (Fig. 3 a, b ; Supplementary Fig. 3a ). However, Rag2 −/− mice treated with AOM-3DSS developed even fewer polyps compared with WT mice (Supplementary Fig. 3k, l ), suggesting that these lymphocytes are not the major regulator of the intestinal tumor development in our experimental setting. Dectin-1 signaling directly enhances PGE 2 production in MDSCs As shown in Fig. 3d and Supplementary Fig. 3a , the expression of genes involved in PGE 2 synthesis was upregulated in polyps of AOM-3DSS-treated GF WT mice, but not in GF Clec7a −/− mice. Decreased expression of Ptgs2 in colonic polyps and non-polyp tissues was also observed in Clec7a −/− mice under SPF conditions (Fig. 4a ), and PGE 2 concentration in colonic tissue homogenate was decreased in these mice (Fig. 4b ). Decreased Ptgs2 expression in intestinal polyps was also observed in Apc Min/+ Clec7a −/− mice (Fig. 4c ), and its expression was only detectable in CD45 + leukocytes, but not in EpCAM + epithelial cells, in both polyps and non-polyp tissues (Fig. 4d ). Fig. 4: Dectin-1 signaling activates the expression of genes involving PGE 2 synthesis. a , b WT and Clec7a −/− mice under SPF conditions were treated with AOM-3DSS for 16 weeks. The expression of Cox2-encoding Ptgs2 was determined by RT-qPCR ( a , WT n = 3, Clec7a −/− n = 5; ** P = 0.0030), and the concentration of PGE 2 in tissue homogenates was determined by ELISA ( b , WT n = 10, Clec7a −/− n = 9; pooled data from 2 experiments and normalized by the protein concentration in each lysate; ** P = 0.0057, * P = 0.0449). c , d The expression of Ptgs2 in intestinal polyp or non-polyp tissues ( c , *** P = 0.0007), or in EpCAM + epithelial cells and in tissue-infiltrating CD45 + leukocytes ( d , *** P = 0.0008, **** P < 0.0001) from Apc Min/+ and Apc Min/+ Clec7a −/− mice at 20 weeks old was determined by RT-qPCR ( n = 3/group). e – g According to the scRNA-seq data shown in Fig. 3e–h , Ptgs2 expressing cells in all polyp-infiltrating myeloid cells ( e ) and Ptgs2 expression levels in Ptgs2 + myeloid cells ( f , WT n = 1284, Clec7a −/− n = 635; **** P < 0.0001) in WT and Clec7a −/− mice are shown. The expression of indicated genes including myeloid subtype-specific genes and PGE 2 synthase genes in WT mice are shown in g . h C57BL/6J mice were treated with AOM-3DSS for 12 weeks. CD11c + and CD11c – CD11b + cells were purified from colonic polyps and non-polyp tissues with autoMACS, and the mRNA expression of indicated genes was determined by RT-qPCR ( n = 4 biologically independent samples/group; *** P = 0.0003, **** P < 0.0001). i Purified CD11b + polyp-infiltrating cells from Apc Min/+ mice were harvested and were stimulated with curdlan for 20 h. Then, the expression of genes involved in PGE 2 synthesis was determined by RT-qPCR. Laminarin treatment was carried out for 4 h before the treatment with curdlan ( n = 4 biologically independent samples/group, **** P < 0.0001). j CD11b + and CD11c + myeloid cells from colonic polyps of AOM-3DSS-treated WT mice were stimulated with curdlan (1 mg/ml) in the presence of each one of inhibitors against IκBα (BAY11-7082, 2 μM)) or SYK (R406, 2 μM). After 20 h, PGE 2 synthase expression was determined by qPCR ( n = 3 biologically independent samples/group; * P = 0.0380, ** P = 0.0037, **** P < 0.0001). Data in a , c , d , h – j are representatives of two independent experiments and are expressed as means ± SD. Data in a – d , h are analyzed using two-way ANOVA followed by Tukey’s multiple-comparisons test, in f using unpaired two-tailed Student’s t -test, and in i , j using one-way ANOVA followed by Tukey’s multiple-comparisons test. Source data are provided in the Source Data file. Full size image By utilizing scRNA-seq analysis on polyp-infiltrating myeloid cells, we found that Ptgs2 and Clec7a was highly expressed in Arg2 + S100a9 + MDSCs (Fig. 4 e, g ). Since MDSC population was decreased in Clec7a −/− mice, Ptgs2 + cell population was also decreased in mutant mice. We also found that Ptgs2 expression levels in myeloid cells were lower in Clec7a −/− mice than that in WT mice (Fig. 4f ). The expression of other PGE 2 synthase genes such as Pla2g6 , Pla2g7 , Ptges1-3 and Ptgs1 was also observed in MDSCs at high levels (Fig. 4g ). MDSCs also expressed Nos2 and Vegfa at high levels. Similar results were also obtained by reanalyzing a public NCBI GEO dataset (GSE196054, scRNA-seq) of intestinal polyp-infiltrating CD45 + leukocytes from AOM-3DSS-treated C57BL/6 mice (Supplementary Fig. 4a–c ). Consistent with this analysis, we found the major enzymes involved in PGE 2 -synthesis were preferentially expressed in tumor-infiltrating CD11c – CD11b + MDSCs but not in CD11c + DCs from AOM-3DSS-treated mice (Fig. 4h ). When polyp-infiltrating CD11b + cells from Apc Min/+ mice were treated with curdlan, the expression of Ptges3 , Ptgs1 , and Ptgs2 was significantly enhanced, and the induction was inhibited by laminarin (Fig. 4i ). Treatment of polyp-infiltrating leukocytes with curdlan also induced PGE 2 synthases both at the mRNA and protein levels (Supplementary Fig. 4d–f ), indicating that Dectin-1 signaling directly induces PGE 2 synthesis in intestinal tumor-infiltrating MDSCs. Previously, we and others showed that Dectin-1 induces cytokines through activation of Syk-CARD9-NF-κB pathway [37] , [38] . Furthermore, COX2 is suggested to be induced by NF-κB p65 [39] , [40] , [41] . Thus, we examined the roles of the Syk-NF-κB pathway in the Dectin-1-induced PGE 2 -synthesizing-enzyme expression. As shown in Fig. 4j , Ptges3, Ptgs1 and Ptgs2 expression were suppressed by the inhibitors against NF-κB (IκBα: BAY11-7082) and SYK (R406), suggesting that these PGE 2 -synthesizing enzymes are induced by the activation of the Dectin-1-Syk-NF-κB pathway. As PGE 2 levels were reduced in Clec7a −/− mouse colon, we examined the effect of PGE 2 on intestinal tumorigenesis. DSS-treated Apc Min/+ Clec7a −/− mice were i. p. administered with PGE 2 every other day for 4 weeks, and colorectal tumor development was examined. As shown in Fig. 5 a, b , colorectal polyp number was increased to the similar level of that in Apc Min/+ mice. Infiltration of MHC-II + CD11c + DCs was decreased, whereas that of MHC-II − CD11b + Ly6C + /Ly6G + MDSCs was increased in polyps after PGE 2 -administration (Fig. 5c ; Supplementary Fig. 4g, h ). The expression of MDSC marker genes such as Itgam , S100a9 , and Clec4e , and tumor proliferation-associated genes, Ccnd1 (Cyclin D1) and Myc (c-Myc), was enhanced after PGE 2 -administration (Fig. 5d ), indicating that MDSC expansion and tumor growth are promoted by PGE 2 . When intestinal polyp-infiltrating cells were treated with PGE 2 in vitro, the expression of these MDSC-associated genes was increased, indicating that these genes were directly induced by PGE 2 (Fig. 5e ). Fig. 5: Oral administration of laminarin inhibits colorectal tumorigenesis, while PGE 2 treatment enhances tumor development. a – d Apc Min/+ Clec7a −/− mice ( n = 3) at 8 weeks old were treated with 2% DSS for 1 week, followed by i.p. injection of PGE 2 (40 μg/mouse) or PBS every other day for 4 weeks. After sacrifice, colorectal polyp development was examined ( a , b ; *** P = 0.0006, ** P = 0.0085). Populations of MHC-II + CD11c + DCs and MHC-II – CD11b + Ly6C + /Ly6G + cells in polyps were determined by flow cytometry ( c ; * P = 0.0193, *** P = 0.0009). Expression of indicated genes in colonic polyps was examined by RT-qPCR ( d ; in Itgam panel, * P = 0.0463; in Clec4e panel, ** P = 0.0084; in Ccnd1 panel, * P = 0.0414; in Myc panel, ** P = 0.0043) ( n = 3/group). e Tumor-infiltrating cells from Apc Min/+ mice ( n = 2) were collected and they were pooled. Then, cells were stimulated with PGE 2 for 20 h, and indicated gene expression was determined by RT-qPCR. Data are the means ± SD of 3–4 wells (* P = 0.0463, *** P = 0.0010, **** P < 0.0001). f – i C57BL/6J mice were administrated with AOM and were treated with 5% laminarin-containing powder food for 10 days each from 3 days before the start of DSS-treatment for 3 cycles. On week 11 after AOM injection, mice were sacrificed and the gross histology of the colon ( f ) and colorectal polyp number of indicated size ( g ; 1–2 mm, * P = 0.030; >2 mm, * P = 0.0334; Total, * P = 0.0452) were examined. The concentration of PGE 2 in tissue homogenate was determined by ELISA ( h , normalized by protein concentration of each lysate; *** P = 0.0006), and mRNA expression of Itgam (CD11b) was examined by RT-qPCR ( i ; Non-polyp, * P = 0.0174; Polyp, *P = 0.0211) ( n = 7/group). Data in a – d , f – i are representatives of two, and in e are representatives of three independent experiments. Data in b – e , g – i are expressed as means ± SD. Data in b , e are analyzed using one-way ANOVA followed by Tukey’s multiple-comparisons test, in c , d , g using unpaired two-tailed Student’s t -test, and in h , i using two-way ANOVA followed by Tukey’s multiple-comparisons test. Source data are provided in the Source Data file. Full size image Administration of laminarin suppresses the development of intestinal polyps To examine therapeutic effects of Dectin-1-blockade on intestinal tumorigenesis, AOM-treated WT mice were fed with 5% laminarin-containing food during 3 cycles of DSS-treatment. Consistent with the observations in Clec7a –/– mice, significantly fewer colorectal polyps developed in laminarin-containing-food-fed mice compared to normal-food-fed mice (Fig. 5 f, g ). Blocking Dectin-1 signaling suppressed intestinal PGE 2 production (Fig. 5h ), accompanied with the reduction of CD11b gene ( Itgam ) expression (Fig. 5i ). These results suggest that Dectin-1 signaling facilitates intestinal tumor development by enhancing PGE 2 , which promotes MDSC expansion. IL-22BP is critically involved in the suppression of tumor development in Clec7a −/− mice We showed that the expression of Il22ra2 was drastically upregulated in polyps of AOM-3DSS-treated GF Clec7a −/− mice (Fig. 3a ; Supplementary Fig. 3a , 5a ), and IL-22BP levels were also increased in AOM-3DSS-treated SPF Clec7a −/− mice (Supplementary Fig. 5b , c ). The expression of Il22ra2 mRNA was also enhanced in both polyps and non-polyp tissues in Apc Min/+ Clec7a −/− mouse intestine (Fig. 6a ). However, gene expression levels of IL-22 and IL-18, the ligand and the regulator of IL-22BP [30] , respectively, were not changed in either AOM-3DSS-treated GF Clec7a −/− or Apc Min/+ Clec7a −/− mice from the Clec7a +/+ counterparts (Fig. 6a ; Supplementary Figs. 3a and 5a , d ). Fig. 6: Il22ra2 expression is highly enhanced in Clec7a −/− mice and deficiency of Il22ra2 aggravates intestinal tumor development in Apc Min/+ Clec7a −/− mice. a Apc Min/+ and Apc Min/+ Clec7a −/− mice were sacrificed at 20 weeks old, and expression levels of Il22ra2 and Il18 in intestinal polyps and non-polyp tissues were determined by RT-qPCR ( Apc Min/+ n = 3; Apc Min/+ Clec7a −/− n = 4; ** P = 0.0078, * P = 0.0148). b Correlations between Il22ra2 and Ptgs2 expression levels in colorectal polyps from GF or SPF mice after treatment with AOM-3DSS are shown ( n = 8/GF, n = 11/SPF group). c In the experiment described in Fig. 5a–d , expression of Il22ra2 in colonic polyps was examined by RT-qPCR after PGE 2 in vivo treatment ( n = 3/group, * P = 0.0261). d Tumor-infiltrating cells pooled from Apc Min/+ mice were harvested and were stimulated with PGE 2 for 20 h, followed by the measurement of Il22ra2 expression by RT-qPCR ( n = 3 biologically independent samples/group; **** P < 0.0001). e Clec7a −/− mice were treated with AOM-3DSS and were sacrificed after 12 weeks of AOM administration. Indicated types of cells in polyps and non-polyp tissues were purified with autoMACS and Il22ra2 expression was examined by RT-qPCR ( n = 3 biologically independent samples/group). f CD11c + cells and CD11c – CD11b + cells were purified with autoMACS, and Il22ra2 expression in these subsets was examined by RT-qPCR ( n = 3 biologically independent samples/group; **** P < 0.0001, *** P = 0.0007). g Polyp-infiltrating cells were prepared from Apc Min/+ mice, and intracellular IL-22BP expression was examined in three indicated myeloid-cell populations by flow-cytometry. Colored numbers in IL-22BP panel represent mean fluorescence intensity. h The experiment described in Fig. 5f was carried out, and 16 weeks after the AOM-DSS-treatment, mean fluorescence intensity (MFI) of IL-22BP expression in MHC-II + CD11c + DCs in colorectal polyp and non-polyp tissues was determined by flow cytometry ( n = 4/group; * P = 0.0121, ** P = 0.0016). i WT mice were administrated with 5% laminarin in diet from 3 days before 1.5% DSS treatment and continued for 7 days until the end of DSS treatment. During DSS-treatment, mice were also i.p. injected with PGE 2 every other day for 4 times. One day after the last PGE 2 injection, mice were sacrificed and MFI of IL-22BP expression in MHC-II + CD11c + DCs was determined by flow cytometry ( n = 3/group; ** P = 0.0035, * P = 0.02323). j Survival rates of indicated mice are shown ( Apc Min/+ n = 19; Apc Min/+ Clec7a −/− n = 66; Apc Min/+ Clec7a −/− Il22ra2 +/− n = 8; Apc Min/+ Clec7a −/− Il22ra2 −/− n = 8; **** P < 0.0001, *** P = 0.0003, * P = 0.0179). k Representative pictures of the small intestine of Apc Min/+ and Apc Min/+ Clec7a −/− mouse of 20 weeks old and Apc Min/+ Clec7a −/− Il22ra2 −/− mouse of 15 weeks old are shown. l Total polyp number in the intestine of Apc Min/+ ( n = 3), Apc Min/+ Clec7a −/− ( n = 3), and Apc Min/+ Clec7a −/− Il22ra2 −/− ( n = 3) mice are shown (* P = 0.0125). m In the scRNA-seq analysis described in Fig. 3e–h , the expression levels of Il22ra2 were determined in each colorectal polyp-infiltrating DC subset. n As in m , RA synthase expression levels in TADC from WT and Clec7a −/− mice were determined by scRNA-seq. o CD11b + and CD11c + cells isolated from WT mouse colon were treated with 10 μM PGE 2 for 20 h, and expression levels of genes encoding RA synthases were examined by RT-qPCR ( n = 3 biologically independent samples/group; Aldh1a3 , * P = 0.0340; Aldh3b1 , * P = 0.0261; Aldh4a1 , * P = 0.0472; Aldh6a1 , ** P = 0.0023). p CD11b + and CD11c + cells isolated from WT mouse colon were treated with indicated doses of PGE 2 (μM) and RA (μM) for 20 h, and expression level of Il22ra2 was examined by RT-qPCR ( n = 3 biologically independent samples/group; * P = 0.030). Data in a , c – l , o , p are representatives of two independent experiments, and in a , c , d – f , h , i , l , o , p are expressed as means ± SD. Data in a , f , h , i are analyzed using two-way ANOVA followed by Tukey’s multiple-comparisons test, in b using Pearson’s correlation coefficient ( r ) test, in c , o using two-tailed Student’s t -test, in d , l , p using one-way ANOVA followed by Tukey’s multiple-comparisons test and in j using Mantel-Cox log-rank test. Source data are provided in the Source Data file. Full size image Interestingly, we noticed that COX2 mRNA levels were negatively correlated with the Il22ra2 expression in colonic polyps under both GF and SPF conditions (Fig. 6b ). Furthermore, Il22ra2 expression in intestinal tumors or IL-22BP expression in myeloid cells was suppressed by PGE 2 treatment both in vivo and in vitro (Fig. 6 c, d ; Supplementary Fig. 5e, f ), suggesting that IL-22BP production is negatively regulated by PGE 2 . To identify Il22ra2 -expressing cells in the intestine, we purified EpCAM + epithelial cells and CD45 + leukocytes from intestinal polyps and found that Il22ra2 mRNA was expressed only in CD45 + but not in epithelial cells (Supplementary Fig. 5g ). Il22ra2 was exclusively detected in CD11b + and CD11c + myeloid cells, but not in Thy1.2 + T cells, CD19 + B cells or other CD45 + cells in both colonic polyp and non-polyp tissues (Fig. 6e ), and its expression was mainly detected in CD11c + DCs, but not in CD11c – CD11b + or other myeloid cells (Fig. 6f ). By flow cytometry, IL-22BP protein was detected in both CD11b – CD103 + CD11c + and CD11b + CD103 int CD11c + DCs, but not in CD11b + CD11c – cells (Fig. 6g ). IL-22BP levels in MHC-II + CD11c + DCs detected by FACS were increased in both polyps and non-polyp tissues after treatment with 5% laminarin in diet during DSS-treatment (Fig. 6h ). Furthermore, co-administration of PGE 2 impaired this laminarin-induced IL-22BP upregulation (Fig. 6i ). Since IL-22BP was reported to play an important role in the suppression of intestinal tumor development [30] , we next examined the role of IL-22BP in the development of intestinal tumors by introducing Il22ra2 −/− mutation into Apc Min/+ Clec7a −/− mice. We found that the life span of Il22ra2 −/− Apc Min/+ Clec7a −/− mice was much shorter than that of Apc Min/+ Clec7a −/− mice, and the life span of heterozygous Il22ra2 +/− mice was still shorter than that of Il22ra2 +/+ Clec7a −/− mice (Fig. 6j ). The polyp number in Il22ra2 −/− Apc Min/+ Clec7a −/− mice of younger age was larger than that in Apc Min/+ Clec7a −/− mice (Fig. 6 k, l ). These results suggest that increased Il22ra2 expression is important for the suppression of intestinal tumor development. Il22ra2 expression was not affected by the treatment with Dectin-1 ligands (Supplementary Fig. 5h ), suggesting that IL-22BP expression is not directly regulated by Dectin-1-signaling. IL-18 has been reported to suppress IL-22BP expression [30] . We found that PGE 2 -induced suppression of Il22ra2 expression was rescued by the treatment with anti-IL-18 antibody (Supplementary Fig. 5i ), suggesting that PGE 2 -induced IL-18 is responsible for the suppression of IL-22BP expression. Actually, Il18 mRNA expression was upregulated in intestinal CD11b + and CD11c + cells after PGE 2 stimulation (Supplementary Fig. 5j ), although its expression level in whole polyp or non-polyp tissues from WT and Clec7a −/− mice were similar (Supplementary Fig. 5a ). Retinoic acid (RA) is also reported to enhance IL-22BP production [42] , [43] and the expression of enzymes involving RA synthesis such as Adh1 and Aldh1a1 was enhanced in polyps in Clec7a −/− mice (Supplementary Fig. 5k, l ). By scRNA-seq analysis, we found a group of DCs, which we named tumor-associated DC (TADC) because this DC subset uniquely expresses tumor-associated genes such as Pclaf , Spc 24 and Top2a (Supplementary Fig. 3d ), highly expressed Il22ra2 in Clec7a −/− mice but not in WT mice (Fig. 6m ). The expression of these Aldh and A / Rdh family genes was highly observed in Clec7a −/− TADCs but not in WT cells (Fig. 6n , Supplementary Fig. 5m ). Since PGE 2 was reported to suppress retinal dehydrogenases (RALDH) expression in both mouse and human DCs [44] , we examined the effect of PGE 2 on the expression of RA-synthase genes in colonic CD11b + and CD11c + myeloid cells, and found that PGE 2 suppressed Aldh , but not A / Rdh , family gene expression (Fig. 6o ; Supplementary Fig. 5n ). When RA was added to colonic or splenic myeloid cells, Il22ra2 expression was significantly recovered (Fig. 6p ; Supplementary Fig. 5o ). These results suggest that PGE 2 controls IL-22BP expression by regulating IL-18 expression and RA production. Dectin-1 signaling enhances PGE 2 synthesis in CRC patients To evaluate the effects of Dectin-1 signaling on CRC development in humans, we firstly examined CLEC7A expression in CRC patients. We found that post-surgery survival rate of patients with high levels of CLEC7A expression (relative expression levels>2, compared with GAPDH ) was significantly lower than those with low levels of CLEC7A expression (<2) (Fig. 7a ). We also noticed that CLEC7A expression levels were positively correlated with the clinical stage of the disease (Fig. 7 b, c ). Disease progression rates were relatively decreased in CRC patients with CLEC7A mutation(s), although the tendency was not statistically significant due to the small number of CRC patients with mutant CLEC7A in TCGA database (Supplementary Fig. 6a ). These observations suggest that DECTIN-1 signaling in humans also correlated with CRC development. Actually, we detected high levels of DECTIN-1 expression on CRC-infiltrating cells, while DECTIN-1-expressing cells were rarely detected in human non-tumor tissues (Fig. 7d ). Fig. 7: The expressions of PGE 2 -synthesizing enzymes and IL22RA2 are modified in CRC patients. a – c Specimens from 36 CRC patients were collected and the post-surgery survival rates of the patients with CLEC7A mRNA expression <2 ( n = 12) or >2 (2–20) ( n = 24) (normalized by GAPDH ) in tumor tissues are shown ( a ). The correlation between CLEC7A expression levels and tumor TNM stage ( b , n = 13 in Stage II, n = 12 in Stage III, n = 8 in Stage IV), and the correlation between the proportion of patients with CLEC7A expression >2 in each stage ( c , n = 13 in Stage II, n = 12 in Stage III, n = 8 in Stage IV) are shown. Tumor TNM stage was determined according to the individual clinical information. In boxplot ( b ), the central horizontal line shows the median; the upper and lower bounds of box show third and first quartile; the upper and lower horizontal lines show the maxima and minima of the data. d Immunohistochemical staining of human Dectin-1 in tumor and non-tumor colon tissues in CRC patients. Green arrows show Dectin-1 + cells. Representative photos from two independent experiments containing nine samples of eight patients are shown. e Specimens from total 68 CRC patients were collected including 23 pairs of tumors and non-tumor specimens from the same individuals. IL22RA2 and PTGS2 expression in tumors and non-tumor tissues were examined by RT-qPCR ( n = 47 in tumor group, n = 44 in non-tumor group; ** P = 0.0084). f Twenty-three pairs of tumor and non-tumor specimens from the same individual were collected, and IL22RA2 and PTGS2 expression were examined ( n = 23/group; ** P = 0.0067, * P = 0.0179). g Correlations of the expression (normalized by GAPDH ) between PGE 2 synthesizing enzymes and CLEC7A in CRC tissues ( n = 47/group). h Pseudotime/trajectory analysis was carried out by using a scRNA-seq dataset (GSE178318) of CRC-infiltrating myeloid cells, in which fully differentiated DCs were excluded. Cell states and their annotations (left panel), and kinetics of relative expression levels of MDSC and macrophage-associated gene markers along the MDSC ‘differentiation’ pseudo-time (right panels) are shown. TAM: tumor-associated macrophage; Mono-DC: monocyte-derived DC. i , j Tumor and non-tumor tissue-infiltrating cells were collected from CRC patients and were stimulated with curdlan for 20 h. In the case of laminarin treatment, cells were first treated with laminarin for 4 h, then curdlan was added to the culture. Expression of PGE 2 synthesizing enzymes ( i ; PTGS2 , 1st *** P = 0.0001, 2nd *** P = 0.0004; PTGES , *** P = 0.0001, **** P < 0.0001) and CD33 ( j ; **** P < 0.0001) was determined by RT-qPCR. Data are the means ± SD of 3 wells. k Tumors from CRC patients were collected and after mincing, small pieces were cultured in the presence of PGE 2 for 20 h. The expression of indicated genes was determined by RT-qPCR. Data are the means ± SD of 3 wells ( HLA-DRA , * P = 0.0122; CD33 , ** P = 0.0033; ITGAM , *** P = 0.0004; IL22RA2 , ** P = 0.0018). l Human PBMCs were harvested from healthy volunteers and were treated with curdlan and celecoxib at the indicated doses in the presence of rGM-CSF + IL-6. After the culture for 5 days, indicated cell number was determined by flow cytometry and was normalized with the average number in control (curdlan 0) group. m In the experiment described in l , after the culture, proportions of whole T cells and CD8 + T cells were determined by flow cytometry. Data in i – k are representatives of three, and in l , m are representatives of two independent experiments and are expressed as means ± SD. Data in a are analyzed using Mantel-Cox log-rank test, in b , c using Spearman rank correlation test, in e using two-tailed Student’s t -test, in f using Wilcoxon matched-pairs signed rank test, in g using Pearson’s correlation coefficient ( r ) test, and in i , j , k using one-way ANOVA followed by Tukey’s multiple-comparisons test. Source data are provided in the Source Data file. Full size image To examine whether the Dectin-1-PGE 2 -IL-22BP axis discovered in mice also exists in humans, we measured the IL22RA2 and COX2 mRNA in tumors from CRC patients. We found that the IL22RA2 mRNA was decreased, while PTGS2 mRNA was significantly increased in tumors compared with non-tumor tissues (Fig. 7e ). This tendency was clearer when samples from the same individuals were compared in a pairwise way (23 pairs of tumor and non-tumor tissues) (Fig. 7f ). We observed that CLEC7A expression was positively correlated with PLA2G2A , PTGS2 or PTGES expression in CRC patients (Fig. 7g ; Supplementary Fig. 6b ). By analyzing the public data on TCGA, we also found that CLEC7A expression was correlated with PTGS2 , PTGES and PTGES3 in CRC patients (Supplementary Fig. 6c ). To confirm Dectin-1-expressing cell profiles and correlation between Dectin-1 and PGE 2 synthases in human CRCs, we carried out scRNA-seq analysis by using pooled cell sequence datasets from six CRC patients (GSE178318) [45] . CRC-associated cells contained lymphocytes, NK, myeloid-derived cells, mast cells, fibroblasts, epithelial, endothelial, and tumor cells, and CLEC7A was mainly expressed in myeloid-derived cells (Supplementary Fig. 7a , b ). We then extracted CLEC7A + myeloid cells, and after re-clustering, we found that the majority of CLEC7A -expressing cells were S100A9 + MDSCs, and less proportion was expressed in CD68 + macrophages and FCER1A + DCs (Supplementary Fig. 7c ). When we further extracted CLEC7A + or – PTGS2 + populations, we found that the average expression level of PTGS2 was significantly higher in CLEC7A + population compared with CLEC7A – ones, especially in MDSCs (Supplementary Fig. 7d ). In CLEC7A + population, PTGS2 expressing cells were largely overlapped with CLEC4E + / S100A9 hi MDSCs and only small number of CD68 hi APOE + macrophages, HLA-DQB1 hi FCER1A + DCs and FCGR3A + monocytes also expressed PTGS2 (Supplementary Fig. 7e ). Other PGE 2 synthase genes such as PTGS1 and PTGES3 were also substantially expressed in CLEC7A -expressing MDSC, DC and macrophage clusters (Supplementary Fig. 7f ). To further analyze the potential link between Dectin-1, MDSC and PGE 2 synthase in human CRC, we carried out pseudo-time/ trajectory analysis by using myeloid-cell population excluding fully differentiated DCs (Supplementary Fig. 7g, h ). After performing the unsupervised simulation, we found that CD68 hi APOE hi HLA-DRA hi tumor-associated macrophages (TAM) and CD68 int APOE int FCGR3A + monocytes ‘differentiate’ into CD68 lo APOE lo HLA-DRA lo CLEC4E hi S100A9 hi MDSCs along the pseudo-temporal trajectory (Fig. 7h left panel). At the same time, we found that in this MDSC ‘differentiation’ process, expression of CLEC7A was gradually upregulated, accompanied with the gradual upregulation of MDSC marker S100A9 and CLEC4E , and with the downregulation of macrophage marker APOE and CD68 . The expression of IL1B , IL6 and PTGS2 were drastically increased for over 10-100 times from the baseline (Fig. 7h ), indicating that these MDSC-promoting factors are induced in the process of MDSC ‘differentiation’, and finally highly expressed by MDSC itself. Different from mouse tumor-infiltrating MDSCs, the expression of ARG1 and NOS2 was not detected in MDSCs (or in any types of tumor-infiltrating leukocytes, Supplementary Fig. 7i ) from CRC patients, but the expression of other functional genes, like IL10 and VEGFA that facilitate tumor development, was upregulated in the process of MDSC ‘differentiation’ (Supplementary Fig. 7i ). To confirm these results, we analyzed another scRNA-seq dataset of CRC patients from GEO (GSE146771), and found that the transcription levels of VEGFA were also in parallel with S100A9 , PTGS2 and CLEC7A in pseudotime-trajectory (Supplementary Fig. 7j ), although the expression of neither ARG1 nor NOS2 was detectable (in MDSCs or in any other leukocytes). When CRC tissues or cancer-infiltrating leukocytes were treated with curdlan, expression of PGE 2 synthase genes was induced in vitro (Fig. 7i ; Supplementary Fig. 6d ). Furthermore, curdlan also upregulated the expression of CD33, a marker of human MDSCs [46] , in both tumor and normal tissues (Fig. 7j ; Supplementary Fig. 6e ), suggesting that Dectin-1 signaling also promotes human MDSC differentiation in CRCs. To further confirm this, we stimulated peripheral blood mononuclear cells (PBMCs) from healthy volunteers with curdlan under MDSC differentiation conditions. After 5 days, MHC-II – CD33 int CD15 + PMN-MDSCs were increased, while MHC-II + CD14 + antigen presenting cells and CD8 + T cells were decreased (Fig. 7 l, m ; Supplementary Fig. 6f ). Addition of COX2 inhibitor partially inhibited the MDSC differentiation and immune cell suppression. Furthermore, the expression of CD33 and CD11B ( ITGAM ) in CRCs was directly induced by PGE 2 and IL22RA2 was suppressed in a dose-dependent manner, suggesting that PGE 2 also promotes MDSC differentiation in humans (Fig. 7k ). By examining the TCGA database, we found that the survival rate of CRC patients with high expression levels of CLEC7A and PTGES was lower than that of low expression group, and that of patients with high expression of IL22RA2 was higher, although the relationship between CLEC7A expression and survival rate was not statistically significant (Supplementary Fig. 6g ). These results suggest that the Dectin-1-PGE 2 -IL-22BP axis is also involved in the regulation of human colorectal carcinogenesis. In the present study, we showed that blocking Dectin-1 signaling suppresses the development of colorectal tumors in both Apc Min familial adenomatous polyposis model and AOM-DSS-induced CRC model. Levels of PGE 2 , which promotes MDSC expansion and tumor development, was reduced in Clec7a −/− mice due to decreased expression of PGE 2 synthesizing enzymes, including Ptgs1 , Ptgs2 , and Ptges3 . In addition, the expression of IL-22BP, which can suppress the development of colorectal tumors by inhibiting IL-22, was significantly increased in Clec7a −/− mice. Furthermore, we found that CRC patients with low CLEC7A expression survive longer compared to those with high expression. A positive correlation was also observed between CLEC7A expression levels and colorectal cancer disease stages. This may be explained by increased infiltration of MDSCs and/or advanced differentiation of MDSCs, which express higher levels of Dectin-1 as indicated by the MDSC trajectory analysis. In CRC patients, IL22RA2 expression was decreased and PTGS2 expression was increased in tumors compared with normal tissues. These observations suggest that Dectin-1 plays important roles in the development of colorectal tumors in both mice and humans, through modification of PGE 2 levels and IL-22BP expression. PGE 2 , a well-known principal mediator of inflammation [47] , plays a critical role in the development of colorectal tumors in AOM-DSS-induced tumor model as well as Apc Min mouse model by binding to the receptor EP2 to enhance the proliferation of tumor cells through induction of genes involved in inflammation and cell growth such as Tnf, Il6 , Cxcl1 , and Cox2 , by activating β-catenin [48] , [49] . Actually, intestinal polyp formation in Apc -deficient mice is suppressed by the Ptgs2 null mutation, and COX-2 inhibitors such as aspirin and other NSAIDs can reduce the incidence and severity of colorectal tumors [50] , [51] . However, the regulatory mechanisms of PGE 2 production have not been elucidated completely. In this study, we showed that deficiency of Dectin-1 impairs the expression of a series of enzymes involved in PGE 2 synthesis, including phospholipase A2 and Cox2, in MDSCs in both AOM-DSS- and Apc Min -induced intestinal tumors. We also showed that Dectin-1 signaling directly induces the expression of these PGE 2 -synthases in tumor-infiltrating MDSCs in vitro. In fact, intestinal levels of PGE 2 were decreased in Clec7a −/− mice, and exogenous PGE 2 administration increased colonic polyposis in Clec7a −/− mice. These results indicate that Dectin-1 signaling promotes intestinal tumorigenesis by enhancing PGE 2 synthesis in MDSCs. Consistent with our observations, previous reports suggested involvement of Dectin-1 in PGE 2 production by the stimulation with β-glucans from yeast [52] , soluble egg antigen from Schistosoma mansoni [53] , and a fungus Paracoccidioides brasiliensis [54] . However, the involvement of this activity in tumorigenesis has not been examined. IL-22BP is a soluble inhibitory receptor for IL-22 [55] , [56] . IL-22BP plays an important role in the regulation of tumorigenesis and its deficiency promotes colorectal tumor development [30] . In the present study, we showed that Il22ra2 disruption enhanced polyp formation in Clec7a −/− mice, consistent with the previous reports. Although we have only compared tumor development between Il22ra2 –/– and Il22ra2 +/+ mice on the Clec7a –/– background, these results suggest that enhanced expression of Il22ra2 in Clec7a –/– mice protects these mice from intestinal tumor development. IL-22BP was produced by intestinal DCs but not by MDSCs. Interestingly, we found that Il22ra2 expression in tumor-infiltrating cells was suppressed by PGE 2 through the suppression of the expression of RA-synthase genes and may also through the induction of IL-18, an inhibitor of Il22ra induction. As PGE 2 concentration was decreased in Clec7a −/− mouse intestine, this finding well explains why Il22ra2 expression was increased in Clec7a −/− mice. Thus, these observations suggest that PGE 2 promotes intestinal tumorigenesis by suppressing Il22ra2 expression as well as by the known tumor enhancing mechanisms of PGE 2 [48] , [49] . In support for this notion, we showed that administrating Clec7a −/− mice with PGE 2 suppressed colonic Il22ra2 expression and abrogated the tumor suppression in Clec7a −/− mice. MDSC accumulation in tumors is considered to enhance cancer progression by promoting invasion of cancer cells, angiogenesis, and metastasis, and inhibiting antitumor immunity [57] , [58] . In this study, we found that both M-MDSC and PMN-MDSC population as well as MDSC-associated gene expression was significantly decreased in colonic polyps of Clec7a −/− mice. In line with our observations, Bhaskaran et al. also reported that Dectin-1-deficiency downregulates MDSC proportion in 4-Nitroquinoline 1-oxide-induced mouse tongue cancer [59] . We showed that proinflammatory cytokine production, such as IL-1β and IL-6, is reduced in Clec7a −/− mice. Rababi et al. also reported that Dectin-1 is critical for the infiltration of Ly6C high monocytes into the inflamed colon and promotes IL-1β secretion through leukotriene B4 production in DSS-colitis model [60] . These myeloid-cell-derived proinflammatory cytokines are important for MDSC differentiation and their growth [28] , [29] . Trajectory analysis also suggest differentiation of macrophage and monocyte population into MDSCs. Furthermore, we showed that Dectin-1 signaling induces production of PGE 2 synthases in MDSCs, and PGE 2 enhances MDSC expansion in mice and in CRC patients. Indeed, we found that Dectin-1 signaling promoted expansion of MDSC population and enhanced their immune-suppressive activity during in vitro MDSC differentiation. Thus, these results indicate that Dectin-1 signaling facilitates MDSC differentiation and expansion by triggering the initiation of an auto-amplification loop, in which Dectin-1 induces inflammatory cytokines in monocytes and macrophages to promote MDSC differentiation and MDSCs produce PGE 2 to further expand themselves. Accumulating evidence suggests that intestinal environment such as commensal microbiota affects development of colorectal tumors. Actually, development of obvious tumors was observed at 16 weeks after AOM-3DSS treatment under SPF conditions, while it took 36 weeks in GF mice in our experimental conditions. In this context, we previously showed that Dectin-1 signaling suppresses the growth of Treg-inducing bacteria such as Lactobacillus and Clostridium species by directly inducing antimicrobial protein calprotectin or by indirectly inducing antimicrobial peptides through induction of IL-17F [11] , [12] , [13] . Thus, blocking Dectin-1 signaling increases colonic Treg cell population in the intestine to suppress mouse colitis [11] , [12] , [13] . In the present study, however, we showed that AOM-3DSS-treated Clec7a −/− mice co-housed with WT mice or Clec7a −/− mice under GF conditions or ABX-treated Apc Min/+ Clec7a −/− mice still developed smaller number of polyps than WT mice, indicating that commensal microbiota are not responsible for the reduced polyp formation in Clec7a −/− mice. Consistent with this notion, Treg cells were not increased in GF Clec7a −/− mice, indicating that Treg cells are not involved in the suppression of polyp formation in Clec7a −/− mouse intestines. Mouse chow used in our experiments contains over 10% of yeast extract, which contains abundant insoluble high MW β-glucans. Our daily diets also contain lots of high MW β-glucans, such as mushrooms and yeasts, as well as low MW β-glucan laminarin from seaweeds. Laminarin is water soluble and contains components with MW less than 5000. These low MW β-glucans are antagonists of Dectin-1 and compete with high MW β-glucans for the binding to Dectin-1 [61] . Many reports suggest that high MW β-glucans can prevent the development of tumors [14] , [15] . In B16 melanoma model, for instance, intraperitoneal administration of high MW β-glucans facilitates antitumor NK cells and cytotoxic T cell responses against tumor cells by activating DCs through Dectin-1 signaling [22] , [23] . Tian et al. also reported that stimulation of monocyte-derive MDSCs isolated from mouse Lewis lung carcinoma with particulate β-glucans promotes the differentiation of these cells into tumor suppressive CD11c + F4/80 + cells and oral administration of these β-glucans promotes antitumor immunity [62] . However, it remains to be explained how orally administered particulate β-glucans are incorporated into blood stream and induce MDSC differentiation in solid tumors. In this study, we showed that oral administration of low MW β-glucan laminarin, but not high MW β-glucans, suppresses colorectal polyposis. Interestingly, Hong et al. tracked β-glucans after oral uptake and found that high MW β-glucans are taken up by macrophages via Dectin-1 and are then degraded into smaller soluble β-glucan fragments [63] . Thus, it is possible that high MW β-glucans are degraded into low MW β-glucans in part after oral administration and inhibit intestinal tumorigenesis by blocking Dectin-1 signaling rather than stimulating it. A recent report identified an additional Dectin-1endogenous ligand, galectin-9 ( Lgals9 ), in pancreatic cancer tissues [25] . In the present study, we showed that galectin-9 expression levels in colonic polyps and non-polyp tissues were similar between WT and Clec7a −/− mice (Supplementary Fig. 3m ), suggesting that β-glucans in food rather than the endogenous ligand is involved in the Dectin-1-dependent regulation of colorectal tumor development. Overall, in this report, we have demonstrated a Dectin-1-mediated colorectal tumor-promoting mechanism, in which β-glucan-induced Dectin-1 signaling promotes PGE 2 production and suppresses anti-tumorigenic IL-22BP expression. Our findings suggest possible influence of daily foods on the development of CRC, and suggest Dectin-1 as a possible target for the prevention and treatment of CRC. Human CRC sample collection Before the collection of human samples from CRC patients, written informed consent was obtained from each patient, and all experiments were carried out following the institutional ethical regulations and guidelines under the protocols approved by the Committee for Clinical Investigation of the First Affiliated Hospital, Sun Yat-sen University (approval number: IIT-2021-654). For tissue-infiltrating cell purification, tumor specimens and/or normal tissue around tumor were cut out and were transferred into ice-cold PBS and placed on ice until use. For the mRNA analysis, we collected 47 tumor specimens and 43 non-tumor specimens from 70 CRC patients, in which 23 pairs of tumor and non-tumor tissues from the same individuals were enrolled. In these patients, we collected the clinical information such as pathological grading, TNM stage, operation and follow-up visiting time of 36 patients, most of whom were followed up around 10 years. Except 12 samples harvested recently, most of the samples were frozen in −80 °C until use for RNA extraction. 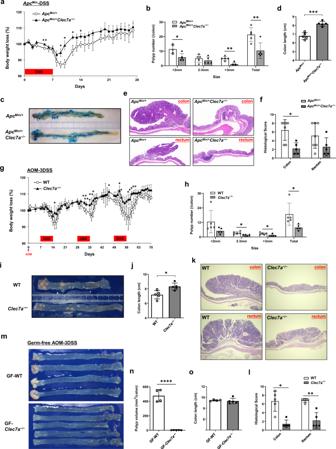Fig. 1: Dectin-1-deficiency suppresses development of colorectal tumors without involvement of commensal microbiota. a–fApcMin/+andApcMin/+Clec7a−/−mice at 8–10 weeks old were treated with 1% DSS for 7 days and were sacrificed 4 weeks later. Body weight changes were observed chronologically after DSS-treatment (a, day5, **P= 0.0098; day9, *P= 0.0297; day10, *P= 0.0127, day12, *P= 0.0260; day14, *P= 0.0364). Number of colorectal polyps with indicated size (b, <2 mm, *P= 0.0130; >3 mm, **P= 0.00139; Total, **P= 0.00948), representative gross pathology of the colon (c) and colon length (d, ***P= 0.00018) are shown (n= 5/group). Representative H.E.-stained histology of the polyps (e) and histopathological scores (f,ApcMin/+n = 7,ApcMin/+Clec7a−/−n = 5; *P = 0.0152) are shown.g–lWT andClec7a−/−mice were i.p. administrated with AOM, and 7 days later, they were treated with 1% DSS for 3 cycles (AOM-3DSS) as described in Methods. Body weight loss was inspected chronologically during the induction of colorectal tumor (g, day15, *P= 0.0352; day32, **P= 0.00129; day35, *P= 0.0237; day36, **P= 0.0088; day37, *P= 0.0338; day46, *P= 0.0475; day52, *P= 0.0339; day53, *P= 0.0179; day57, *P= 0.0290; day58, *P= 0.0276; day59, *P= 0.0119; day60, *P= 0.0251; day61, *P= 0.0196). Mice were sacrificed at week 16 after AOM administration, and number of colorectal polyps with indicated size (h, 2–3 mm, *P= 0.0150; >3 mm, *P= 0.0339; Total, *P= 0.0312), gross pathology of the colon (i), colon length (j, *P= 0.0103), representative histology of the polyps (k) and histopathological scores (l, *P= 0.0159, **P= 0.0079) are shown (n= 5/group).m–oGF WT andClec7a−/−mice were treated with AOM-3DSS. Thirty-six weeks after AOM administration, these mice were sacrificed, and gross pathology of the colon (m) and colon length (o) are shown. Colorectal tumor sizes in indicated mice were measured and total polyp volume (n, ****P< 0.0001) is shown. The polyp volume was calculated as (diameter)3for circular polyps and as (Short diameter)2× (long diameter) for elliptic polyps (n = 4/GF WT group,n= 5/GFClec7a−/−group). Data in (a-f) are representatives of five, ing–lare representatives of six, and inm-oare representatives of three independent experiments. Data ina,b,d,f,g,h,j,l,n,oare presented as means ± SD. Data ina,b,d,g,h,j,n,oare analyzed using unpaired two-tailed Student’st-test and inf,lusing two-tailed Mann–WhitneyU-test. Source data are provided in the Source Data file. Details of patient clinical information including TMN stage, pathological grading, and tumor size are available in Supplementary Table 1 . Mice Clec7a −/− mice were generated as described before [5] and used after backcrossing for 9 generations to C57BL/6 J. Apc Min/+ mice, kindly provided by Dr. Ryo Abe, Tokyo University of Science, were crossed with Clec7a −/− mice to generate Apc Min/+ Clec7a −/− mice. C57BL/6J mice, which were originally purchased from Sankyo Lab Service (Saitama, Japan) for Clec7a −/− mouse backcrossing, and their offspring were maintained in the same animal room as that Clec7a −/− mice were housed and used as the control. GF WT mice were purchased from Sankyo Lab Service. GF Clec7a −/− mice were generated by taking out sterile babies from the uterus of a SPF full-term pregnant female by cesarean section and transferring these babies in the care of 2 to 3 GF WT mothers that were nursing their recently delivered litters in a GF isolator. Age- and sex-matched WT mice were separately housed or co-housed with Clec7a −/− mice after weaning at 4 weeks old. All mice were kept under specific pathogen-free conditions with γ-ray sterilized normal diet (Funakoshi Kagaku, Chiba, Japan), acidified (0.002 N HCl, pH 2.5) tap water, and autoclaved wooden chip bed in environmentally controlled clean rooms at the experimental animal facilities of the Center for Animal Disease Models, Research Institute for Biomedical Sciences, Tokyo University of Science, and of Zhongshan School of Medicine, Sun Yat-sen University. All animal experiments were carried out following the institutional ethical regulations and guidelines and with protocols approved by the Institutional Animal Care and Use Committee of the Tokyo University of Science, and by the Experimental Animal Manage and Use Committee of Sun Yat-sen University (approval number 2020000113, 2021001577). Since both male and female Clec7a −/− mice exhibited the same phenotypes in all disease models in the present study, mice of both genders were used. Generation of Apc Min/+ Clec7a −/− Il22ra2 −/− mice Il22ra2 −/− mice on Apc Min/+ Clec7a −/− background were generated by CRISPR-Cpf1 method. Briefly, the targeting sequence on the mouse Il22ra2 exon 3 with the PAM sequence was determined as (TTTCATTGGTCAGGTCACAGAAGAGCGC), and the guide RNA (crRNA) was obtained from Integrated DNA Technologies (IDT, Coralville, IA, USA). Then 1.2 mM crRNA was mixed with 0.6 mM CRISPR-Cpf1 nuclease (Cat# 1081068, IDT) and was transferred into Apc Min/+ Clec7a −/− zygotes by micro-injection. On the next morning, normal 2-cell stage embryos were transferred into the oviducts of pseudo-pregnant female mice. The genotypes of mutant babies were determined by sequencing the RT-PCR product with the primers ATTTGTGTGTTTTCCCATCCTC (Forward) and TCAAAGGCAGAAGAGAAAAAGG (Reverse). Three mutant mice, all of which had 19 bp deletion that causes a frame-shift and premature termination of IL-22BP, were identified, and one of them was used to generate homozygous Apc Min/+ Clec7a −/− Il22ra2 -deficient mice. Induction of intestinal polyps in Apc Min mice Apc Min/+ or Apc Min/+ Clec7a −/− mice were normally kept under SPF conditions for 19–23 weeks after birth until polyps in small and large intestines develop spontaneously. For the induction of colorectal tumors, same mice at 8–10 weeks old were treated with 1% DSS in drinking water for 1 week, and they were maintained for another 4–5 weeks before sacrifice. Chemical induction of colorectal tumor Six to 7-weeks-old mice were administrated intraperitoneally (i.p.) with 10 μg per gram body weight of AOM (Cat# 011-20171, Wako, Osaka, Japan). One week after the administration, these mice were treated with 1% DSS (36–50 kDa; Cat# 216011090, MP Biomedicals, Illkirch, France) in their drinking water for 7 days followed by 14 days of normal water. After 3 cycles of DSS/normal water-treatment, these mice were further maintained for additional 2–6 weeks before sacrifice. Cell preparation Colonic tumor/ non-tumor tissue-infiltrating cells were prepared as follows. Briefly, tissue pieces were cut into 1 mm slices, then they were shaken for 40 min in Hanks‘ Balanced Salt Solution (HBSS) containing 3 mM EDTA at 37 °C. Intra-epithelial lymphocytes and colonic epithelial cells in the culture supernatant were discarded, and the gut slices were washed twice with HBSS. Then, they were shaken at 37 °C for 120 min in RPMI containing 10% FBS and 1% streptomycin+penicillin, 200 U/ml collagenase (Cat# C2139; Sigma-Aldrich), and 5 U/ml Dnase 1 (Sigma-Algrich). After the incubation, the samples were vortexed for 10 s, and single-cell suspension was harvested after sterile gauze-filtration. To prepare lymphocytes, tissue-infiltrating cells were further purified on a 45%/66.6% discontinuous Percoll (Cat# 17-0891-01, Cytiva Life Sciences) gradient at 2200 rpm for 20 min. Cell and tissue in vitro culture Tissue-infiltrating cells (2 × 10 5 ) from mouse/ human colorectal tumors or non-tumor tissues, or mouse/ human colorectal tumor pieces or non-tumor tissue pieces (3 × 3 mm), were cultured in a 0.2 ml RPMI containing 10% FBS and 1% streptomycin plus penicillin at 37 °C under 5% CO 2 in a 96-well flat-bottomed plate (Falcon, Becton Dickinson). To induce MDSC differentiation in vitro, mouse bone marrow cells or human PBMCs were harvested from thigh and shin bones of mice or peripheral blood of healthy volunteers, respectively, and were cultured with recombinant mouse GM-CSF and IL-6 (Cat# 315-03, 216-16, Peprotech Inc., Rocky Hill, NJ, USA) in 48-well flat-bottomed plate (Falcon) for 120 h. For T cell activation, CD4 + or total T cells were isolated from the spleen, and were cultured with the stimulation of anti-CD3/CD28 Dynabeads (Cat# 11456D, Thermo Fisher Scientific) for 3-4 days. In some experiment, anti-mouse IL-18 antibody (Cat# 210-401-323, Rockland Immunochemicals, Inc, Philadelphia, PA, USA) was added to the culture with or without PGE 2 stimulation. In other experiments, inhibitors of NF-κB (IκBa: BAY11-7082, Cat# SF0011, Beyotime, China) or SYK (R406, Cat# SC1022, Beyotime) was added to the culture after stimulation with curdlan. After the culture, cells or tissues were collected and mRNA expression was measured by quantitative reverse transcription PCR (RT-qPCR) or cell population was examined by flow cytometry. Purification of epithelial cells and immune cells from lamina propria Cells from mouse whole intestines or from polyps were labeled with biotin-conjugated anti-mouse CD326/EpCAM (G8.8) (Cat# 118203, Biolegend), followed by microbeads-conjugated anti-biotin CD326 + epithelial cells were positively sorted by using autoMACS (Miltenyi Biotec, Bergisch Gladbach, Germany). The CD326 negative fraction was then sorted with anti-mouse CD45 (Cat# 130-052-301) microbeads for leukocyte purification, or was sorted with anti-mouse CD11b (Cat# 130-049-601) and CD11c (Cat# 130-125-835) microbeads for myeloid-derived cells. Anti-Thy1.2 (Cat# 130-121-278) microbeads were used for T cells and anti-CD19 (Cat# 130-121-301) microbeads were used for B cell sorting. All the antibody-conjugated microbeads were obtained from Miltenyi Biotec. Colonic polyp-infiltrating myeloid cells for scRNA-seq analysis were stained with anti-mouse CD11b and CD11c antibodies for flow cytometry and were sorted by FACS Aria Fusion (BD Biosciences). Flow-cytometry Antibodies against mouse CD4 (GK1.5, Cat# 100411), CD8α (53-6.7, Cat# 100707), TCRγδ (GL3, Cat# 118105), CD45 (30-F11, Cat# 103115, 103113), CD19 (6D5, Cat# 115505), CD3ε (KT3.1.1, Cat# 155607), Ly6C (HK1.4, Cat# 128007, 128025), Ly6G (1A8, Cat# 127605, 127633), CD11b (M1/70, Cat# 101215), CD11c (N418, Cat# 117321), I-A/I-E (M5/114.15.2, Cat# 107613, 107627), CD103 (2E7, Cat# 121405), IgG1 (RMG1-1, Cat# 406607), NOS2 (W16030C, Cat# 696805), IFN-γ (XMG1.2, Cat# 505805), IL-17 (TC11-18H10.1, Cat# 506917), Foxp3 (MF-14, Cat# 126403), CD326 (G8.8, Cat# 118203), Thy1.2 (30-H12, Cat# 105304) and anti-human CD33 (HIM3-4, Cat# 303303), CD14 (M5E2, Cat# 301807), CD15 (W6D3, Cat# 323005), HLA-DR (L243, Cat# 307645), CD3ε (HIT3a, Cat# 300305) and CD8α (SK1, Cat# 344721) were purchased from Biolegend (San Diego, U.S.A.). Antibody against mouse Dectin-1 (2A11, Cat# ab21646) was purchased from Abcam (Cambridge, UK). Anti-mouse IL-22BP polyclonal antibody was purchased from R&D systems (Cat# IC2376A, Biotechne, Minnesota, U.S.A). 7-AAD (7-amino-actinomycin D) staining solution were obtained from eBioscience (Cat# 00-6993-50, San Diego, CA, USA). The anti-CD16/CD32 (2.4G2, anti-FcγRIII/II) mAb was obtained from Tonbo Biosciences (Cat# 70-0161-U500, San Diego). All antibodies were used at a 1:250 dilution. Cells isolated from mouse intestine were washed twice with FACS Hanks buffer (HBSS containing 2% FCS) and then treated with 2.4G2 to block non-specific FcR binding. Cells were then surface-stained with mAbs for 25-30 min. For the analysis of cytokine expression by FACS, cells were first stimulated with 50 ng/ml PMA (Cat# P8139, Sigma Aldrich) + 500 ng/ml ionomycin (Cat# 407952, Sigma Aldrich) and 1 mM monensin (Cat# 475897, Sigma Aldrich) for 4 h. After the stimulation, cells were washed twice with FACS Hanks buffer and then treated with 2.4G2 to block FcR binding. Cells were then stained with mAbs against cell-surface markers for 30 min and were fixed and permeabilized with Cytofix/Cytoperm solution (Cat# 554722, BD Biosciences) for 20 min. After washing with washing buffer, cells were incubated with anti-mouse IFN-γ and IL-17 mAbs for another 30 min. The fluorescence was detected by a Canto II or FACSCalibur flow cytometer (BD Biosciences) and FlowJo v10.0 & v10.1 software (BD Biosciences) was used for the analysis. Quantitative reverse transcription PCR (RT-qPCR) Total RNA was extracted with a Mammalian Total RNA Miniprep kit (Cat# RTN350-1KT, Sigma Aldrich). RNA was denatured in the presence of an oligo dT primer and then reverse transcribed with a High Capacity cDNA Reverse Transcription kit (Cat# 4368814, Applied Biosystems, San Francisco, U.S.A.). 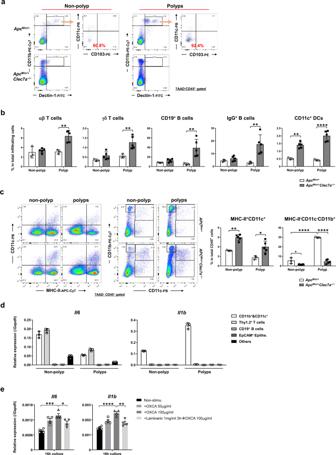Fig. 2: MHC-II+CD11c–CD11b+cell population is decreased in the colon ofClec7a–/–mice. aApcMin/+andApcMin/+Clec7a−/−mice were treated with 1% DSS for 7 days and were sacrificed 4 weeks later. Flow cytometric analysis was carried out to identify Dectin-1-expressing cells in colorectal polyps and non-polyp tissues.b,cApcMin/+andApcMin/+Clec7a−/−mice were treated with 1% DSS for 7 days and were sacrificed 4 weeks later. Proportions of T cells, B cells and DCs in total tissue-infiltrating cells (b, αβT cells, **P= 0.0020; γδT cells, **P= 0.0076; CD19+B cells, **P= 0.0069; IgG+B cells, **P= 0.0058; CD11c+DCs, **P= 0.0014, ****P< 0.0001), and proportions of MHC-II+CD11c+and MHC-II+CD11c–CD11b+cells in tissue-infiltrating CD45+cells (c, MHC-II+CD11c+, **P= 0.0039, *P= 0.0157; MHC-II−CD11c−CD11b+, *P= 0.0563, ****P< 0.0001) in non-polyp tissues or polyps in the colon were examined by flow cytometry (n= 3/ApcMin/+group,n= 5/ApcMin/+Clec7a−/−group).dWT mice were treated with AOM-3DSS and were sacrificed after 12 weeks. Indicated types of cells in polyps and non-polyp tissues were purified with autoMACS andIl6andIl1bexpression was examined by RT-qPCR (n= 3 biologically independent samples/group).eWT mice were administrated with AOM followed by 3 cycles of DSS. After 11 weeks of AOM treatment, these mice were sacrificed and CD11b+and CD11c+cells were purified from colorectal polyps with autoMACS. The sorted cells were stimulated with an agonistic β-glucan OXCA for 16 h with or without pretreatment with an antagonistic β-glucan laminarin, for 3 h, then,Il6andIl1bexpression were determined by RT-qPCR (n= 4 biologically independent samples/group; inIl6panel, ***P= 0.0002, *P= 0.0382;Il1bpanel, ****P< 0.0001, **P= 0.0012). Data ina–eare representatives of two independent experiments. Data inb–eare expressed as means ± SD. Data inb,care analyzed using two-way analysis of variance (ANOVA) and ineusing one-way ANOVA followed by Tukey’s multiple-comparisons test. Source data are provided in the Source Data file. 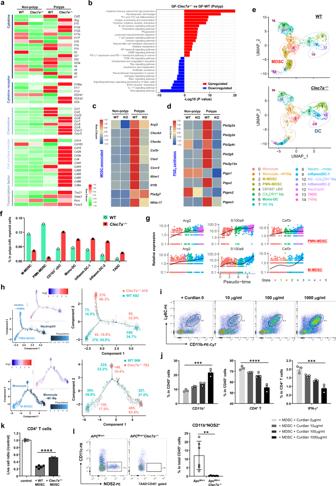Fig. 3: The expression of genes encoding PGE2-synthesizing enzymes and IL-22BP is regulated by Dectin-1 signaling. a–dGF WT andClec7a−/−mice treated with AOM-3DSS shown in Fig.1mwere sacrificed at 36 weeks after AOM administration, and RNA-seq analysis was carried out by using RNAs from polyps and non-polyp tissues in the vicinity (pooled 4 WT and 5Clec7a−/−GF mice). Expression levels of genes for cytokine, chemokine, cell-surface marker, and T cell transcription factor in WT andClec7a−/−mice are shown as heatmaps (a). Cell populations, signaling pathways and metabolic pathways were compared betweenClec7a−/−and WT mouse polyps by using the KEGG database. Log2 (fold-change) > 1 is upregulated genes, while log2 (fold-change) <−1 is downregulated genes (b). Expression levels of MDSC-associated genes are presented as a heatmap (c). Expression levels of PGE2-synthase genes in polyp and non-polyp tissues are shown as a heatmap (d).e–hSPF WT andClec7a−/−mice treated with AOM-3DSS for 16 weeks, and CD11b+and CD11c+cells were purified from colorectal polyps and were applied to scRNA-seq analysis. UMAP showing cell type cluster distribution (e), proportions of MDSC and DC subsets (f), changes of typical MDSC-associated gene expressions during MDSC development (g), and the trajectory tracks of the differentiation of PMN-MDSCs and M-MDSCs (h) in WT andClec7a−/−mice are shown (5 WT and 4Clec7a−/−mice pooled).iBone marrow cells from WT mice were harvested and were stimulated with rGM-CSF and rIL-6 (2 × 105cells/well) for 5 days. Curdlan with indicated doses was added on the 2nd day and flow cytometry was carried out to examine MDSC differentiation by staining with antibodies against Ly6C and CD11b.jAfter the culture ini, differentiated bone marrow cells were further co-cultured with splenic CD4+T cells from WT mice for 2 days in the present of anti-CD3/CD28 microbeads. After the co-culture, proportions of CD11b+and CD4+cells in CD45+cells and the proportion of IFN-γ+cells in CD4+cells were determined by flow cytometry (n= 3 biologically independent samples/group; in CD11b+panel, ***P= 0.0009; in CD4+T panel, ****P< 0.0001; in IFN-γ+panel, ***P= 0.0001).kEpCAM−MHC-II−Gr1+cells were isolated from colonic polyps of AOM-3DSS-treated WT andClec7a−/−mice and were co-cultured with splenic CD4+T cells in the presence of anti-CD3/CD28 microbeads. Two days later, flow cytometry was carried out to determine the number of live CD4+T cells (controln= 3, +WT MDSCn= 5, +Clec7a−/−MDSCn= 3, ****P< 0.0001).lIntestinal polyp-infiltrating cells were isolated fromApcMin/+andApcMin/+Clec7a–/–mice, and proportions of NOS2-producing CD11c–CD11b+cells were determined by flow cytometry (ApcMin/+n= 6,ApcMin/+Clec7a−/−n= 7, **P= 0.0027). Data ini,jare representatives of three and inkis representative of two independent experiments. Data from two independent experiments are pooled inland inj–lare expressed as means ± SD. Data inj,kare analyzed using one-way ANOVA followed by Tukey’s multiple-comparisons test and inlusing unpaired two-tailed Student’st-test. Source data are provided in the Source Data file. qPCR was performed with a SYBR Green qPCR kit (Cat# 639676, Takara Bio., Shika, Japan) and C1000 Thermal Cycler system (Bio-Rad, Hercules, USA) with the sets of primers described in Supplementary Table 2 , and relative mRNA expression levels were calculated with the comparative cycle threshold (Ct value) method and were normalized with Gapdh mRNA expression level. Bulk RNA sequencing and analysis Total RNA was isolated from colorectal tumor or non-tumor tissues using Sigma Aldrich total RNA-prep kit. RNA was prepared using Contech SmartSeq2 library prep kits and sequenced with NovaSeq6000. Data were processed with Galaxy (usegalaxy.org). Quality filtering and adapter trimming of the resulted reads were performed by Trimmomatic [64] , aligned to GRCm38 (mm10) whole-genome data by HISAT2 [65] , assembled to transcripts by StringTie [66] . Data were normalized by total lead count correction and transformed to log2 (TPM + 1) for further analysis. Genes with log2 (fold-change) >1 or <−1 were considered as upregulated and downregulated genes, respectively. Gene with log2 (fold-change) >1 or <−1 was input for KEGG pathway analysis with Benjamini and Hochberg method. P -value <0.05 and q -value <0.1 are considered as significant. Heatmaps were plotted using Tbtools software [67] , and the z -score was calculated by transcripts per million (TPM), as (TPM-average of TPM)/Standard deviation. PGE 2 and IL-1β concentration measurement Polyps and non-polyp tissues from mouse colon were harvested and were put into 2 ml tubes containing 500 μl lysis buffer for protein [RIPA buffer: 50 mM Tris-HCl (pH 8.0) + 100 mM NaCl + 0.1% Triton X-100] and 50 μl protease inhibitor cocktail (Takara Bio, Shika, Japan). Tissue was homogenized with beads and Micro Smasher (MS-100R, TOMY). After centrifugation, supernatant of tissue homogenate was collected and PGE 2 and IL-1β concentration was measured by ELISA Development Kit for PGE 2 (Cat# KGE004B, R&D systems) and ELISA MAX™ Standard Set for IL-1β (Cat# 432601, Biolegend). The concentration of PGE 2 was normalized to total protein concentration of each individual. Antibiotics treatment Apc Min/+ mice were pretreated with an antibiotics (ABX) mixture containing 500 mg/l vancomycin (Cat# V820413), 1 g/l ampicillin (Cat# A6265), 1 g/l metronidazole (Cat# M813526) and 1 g/l neomycin (Cat# N814740) (VAMN, Macklin Inc., Shanghai, China) for 3 weeks with addition of 75 g/l sucrosein drinking water, and then were co-administrated with DSS for 1 week, and were continuously treated with ABX for further 4 weeks. In some experiment, ABX cocktail containing 0.4 g/l kanamycin (Cat# K812216), 0.035 g/l gentamycin (Cat# G6064), 0.0570 g/l colistin (Cat# C805491), 0.215 g/l metronidazole, 0.045 g/l vancomycin HCl and 0.025 g/l erythromycin (Cat# E808820) [68] (6 mixture, Macklin) were used to treat mice. β-glucan treatment Agonistic Dectin-1 ligand curdlan was purchased from Wako Pure Chemical Corp. and NaClO-oxidized Candida albicans (OXCA) was prepared by Prof. Ohno at Tokyo Pharmaceutical University [69] . Colonic polyp or non-polyp-infiltrating cells were treated with curdlan or OXCA for 16 or 20 h, and the expression of cytokine and PGE 2 synthesizing enzyme was examined. Dectin-1 antagonist laminarin (Cat# L9634, 1 mg/ml, Sigma-Aldrich, St. Louis, MO, USA) treatment was carried out for 4 h before curdlan treatment. For laminarin treatment in vivo, mice were firstly i.p. administrated with AOM and then were treated with 5% laminarin (Cat# L0088, Tokyo Chemistry Industry, Tokyo, Japan) mixed in powder food from 3 days before the start of DSS-treatment for 10 days, and this laminarin-DSS treatment were carried out for 3 cycles. PGE 2 treatment PGE 2 was purchased from TopScience Co. Ltd, Shanghai, China (Cat# T5014). For in vitro treatment, colonic polyp or non-polyp-infiltrating cells were treated with PGE 2 (0.1–10 μM) for 20 h, and the expression of myeloid-cell marker genes was examined. For in vivo treatment, mice at 8 weeks old were firstly treated with 2% DSS for 1 week, then were i.p. injected with 40 μg/mouse PGE 2 or PBS every other day for 4 weeks. Single-cell RNA-seq library construction and sequencing After colonic polyp-infiltrating myeloid-derived cells were harvested, cell count and viability was estimated using fluorescence Cell Analyzer (Countstar® Rigel S2) with AO/PI reagent. Fresh cells were resuspended at 1 × 10 6 cells/ml in PBS containing 0.04% bovine serum albumin. Single-cell RNA-Seq libraries were prepared using SeekOne® MM Single Cell 3’ library preparation kit (SeekGene, Cat# SO01V3.1). Briefly, appropriate number of cells were loaded onto the flow channel of SeekOne® MM chip which had 170,000 microwells and allowed to settle in microwells by gravity. After removing the unsettled cells, sufficient C ell B arcoded Magnetic B eads (CBBs) were pipetted into flow channel and were also allowed to settle in microwells with the help of a magnetic field. Next, excess CBBs were rinsed out and cells in MM chip were lysed to release RNA, which was captured by the CBB in the same microwell. Then all CBBs were collected and reverse transcription were performed at 37 °C for 30 min to label cDNA with cell barcodes on the beads. Further Exonuclease I treatment was performed to remove unused primer on CBBs. Subsequently, barcoded cDNA on the CBBs was hybridized with random primer, which had read 2 SeqPrimer sequence on the 5’ end and could extend to form the second strand DNA with cell barcode on the 3’ end. The resulting second strand DNA were denatured off the CBBs, purified and amplified in PCR reaction. The amplified cDNA product was then cleaned to remove unwanted fragment and added to full length sequencing adapter and sample index by indexed PCR. The indexed sequencing libraries were cleanup with SPRI beads, quantified by quantitative PCR (KAPA Biosystems KK4824) and then sequenced on illumina NovaSeq 6000 with PE150 read length. Preprocessing of single-cell RNA-seq data analysis Single-cell sequencing data obtained from the present study or pre-processed data of AOM-3DSS-treated C57BL/6 mice (GSE196054) and CRC patients (GSE178318 [45] and GSE146771 [70] ) from NCBI GEO database were converted into a Seurat object by the R package (version 4.1.3) using the software Rstudio Desktop v2022.02.3 (Posit Software, PBC) and then were filtered to remove cells with a number of unique gene counts over 4000 or less than 200. Cells with more than 5% of mitochondrial gene counts were also filtered. After unwanted cells were removed from the dataset, a global-scaling normalization method “LogNormalize” was carried out to normalize the feature expression measurements for each cell by the total expression, multiply this by a scale factor of 10,000, and log-transform the result. Over 95% of high-quality cells with total more than 25,000 protein-coding genes were remained after the filtering and normalization for the downstream processing. Identification of cell types and gene expression by dimensional reduction After the normalization, subsets of feature genes were calculated that exhibit high cell-to-cell variation in the dataset. Next, a linear transformation (scaling data) and following linear dimensional reduction were performed. Then, cells were clustered by feature gene profiles. The annotation of each cell cluster was confirmed by the expression of canonical marker genes such as: T cells ( CD3D , TRAC ), B cells ( CD19 , MS4A1 ), plasma cells ( JCHAIN , IGHA1 , CD79A ), macrophages ( CD68 , APOE , MERTK ), MDSCs ( S100A8 , S100A9 , CLEC4E , CD33 ), DCs ( FCER1A , CST3 , HLA-DQB1 ), mast cells ( TPSAB1 , MS4A2 ), fibroblasts ( COL1A1 , COL3A1 ), epithelial cell ( EPCAM , KRT8 , KRT18 ) and tumor cells ( TK1 , STMN1 , TUBB ). Analysis for pseudo-temporal trajectory of MDSC differentiation Tumor-infiltrating myeloid cells, in which PTPRC lo non-leukocytes, CD3D + TRAC + T cells and CST3 hi HLA-DRA hi DCs were excluded by Seurat in R, were extracted from scRNA-seq dataset of CRC (GSE196054). Pseudotime/ trajectory analysis for MDSC differentiation was then performed by using the R package Monocle and Monocle3. Simulation of MDSC differentiation that orders myeloid cells along a pseudotemporal trajectory was output through unsupervised Monocle processing. Expression of S100A9 and CLEC4E was used as the differentiation marker for MDSCs and that of CD68 and APOE was used for macrophages. Histopathological analysis Colon and rectum with polyps were removed and fixed with 10% neutral buffered formalin and embedded in paraffin. After being cut into 5 μm slices, tissue sections were stained with haematoxylin and eosin. Histopathological score was evaluated according to a previous report [71] : for number of lesions ( L ), 1 = 0–2, 2 = 3–5, 3 = 6–8, 4 = 9~; for crypts (C): 0 = normal, 1 = goblet cell depletion, 2 = branching, 3 = complex budding; for Epithelium (E): 0 = normal, 1 = hyperplasia, 2 = low-grade dysplasia, 3 = high-grade dysplasia; for Submucosal invasion (S): 0 = absent, 1 = present. The total histological score was calculated as L + C + E + S . Immunohistochemistry (IHC) For immunohistochemistry, tumor and non-tumor tissues from CRC patients after surgery were rinsed with PBS and fixed with 10% formalin. After fixation, tissues were dehydrated in ethanol overnight for paraffin embedding. After paraffin embedding, the paraffin block was cut into 5 μm slices. After deparaffinization, the tissue slices were rehydrated in 3,3′-diaminobenzidine solution and were treated with H 2 O 2 to close the endogenous peroxidase. Then the slices were incubated in retrieval solution at 60 °C overnight for heat-induced epitope retrieval, followed by treatment with 1% BSA for 2 h to block non-specific antibody binding. Then, the slices were incubated with 1 μg/ml of primary antibody against human Dectin-1 (Cat# ab140039, Rabbit polyclonal to human and Rat Dectin-1, Abcam Inc, Cambridge, UK) overnight at 4°C, followed by HRP-conjugated anti-rabbit IgG (Cat# GB23303, Servicebio co. Wuhan, China) for 15 min at room temperature. Tissue slices were then treated with DAB substrate solution for 1-3 min, and with hematoxylin counterstain for additional 10 seconds at room temperature. Photos of IHC were taken by Leica DM6FS with imaging scanning system (Leica Camera AG, Wetzlar, Germany). Western blot analysis For the detection of IL-22BP protein levels in mouse intestinal polyps tissues, a piece of tissue (200 mg) was firstly lysed with 0.1 ml RIPA buffer (25 mM Tris-HCl, pH 7.5, 50 mM NaCl, 0.5% NP-40, 0.1% SDS, 0.5% DOC, 1 mM DTT, 20 mM NEM supplied with fresh Protease inhibitors). A syringe with sonicator was used to mechanically crush the tisuses. For the detection of IL-22BP, PTGES3, COX1 and COX2, in CD11b + and CD11c + cells (1–3 × 10 5 ) isolated from mouse intestinal polyps, after PGE 2 or curdlan stimulation for 20 h, cells were washed with 1 ml PBS and were directly lysed in 100 μl RAPI buffer. Lysate was centrifuged at 12,000 rpm for 30 min at 4 °C. The supernatant was transferred to a new tube and the protein concentration was measured with BCA protein assay kit (Bioteke, Cat# PP1001). The cell lysate was denatured for 10 min at 99 °C in a loading buffer (NuPAGE 4×, Reducing Agent 10×, Beyotime, Cat# P0015L) and was loaded on a ExpressPuls TM 4–20% PAGE Gel (Genscript, Cat# M42012C). After electrophoresis, proteins in the gel were transferred to a PVDF membrane (Millipore, Cat# IPVH00010) for 60 min with 200 mA. PowerPa TM Basic power supply and Mini-PROTEAN Tetra Cell 4-Gel System (Bio-Rad) were used for both electrophoresis and membrane transfer. The membrane was then sunk in a TBST solution (50 mM Tris-Cl, 150 mM NaCl, 0.1% Tween-20) with 5% of non-fat milk (Biofroxx, Cat# 1172gr100), and was then incubated with specific primary antibodies (listed below) overnight at 4°C. In the next morning, the membrane was washed and was incubated with a horseradish peroxidase-conjugated secondary antibody for 1 h. The membrane was then washed, and protein bands on the membrane were visualized by the Pierce TM ECL Western Blotting Substtrate (Thermo, Cat# XA338096) and were detected by Amersham TM Imager 600. Chemiluminescence intensity of each band was calculated by the imaging analysis software ImageJ version 1.53t. Antibodies used: Mouse IL-22BP Antibody (Bio-techne, Cat# AF2376, 0.1 μg/ml) Human/Mouse p23/PTGES3 Antibody (Bio-techne, Cat# MAB100391, 2 μg/ml) Human/Mouse COX-2 Antibody (Bio-techne, Cat# AF4198-SP, 1 μg/ml) Human/Mouse COX-1 Antibody (Bio-techne, Cat# MAB37401, 2 μg/ml) THETM beta-Actin mouse Antibody (GenScript, Cat# A00702-100, 1:3000) HRP-conjugated Affinipure Donkey Anti-Goat IgG (H + L) (Proteintech, Cat# SA00001-3, 1:1000) HRP-conjugated Affinipure Rabbit Anti-Sheep IgG (H + L) (Proteintech, Cat# SA00001-16, 1:1000) Goat Anti-Mouse IgG Antibody (H&L) [HRP], pAb (GenScript, Cat# A00160, 1:3000). Statistical analysis Differences in parametric data were evaluated by the unpaired two-tailed Student’s t -test. For experiments containing more than two relative groups, one-way ANOVA followed by Tukey’s multiple-comparisons test was performed. Statistical significance of survival rate between groups was assessed by the log-rank test. 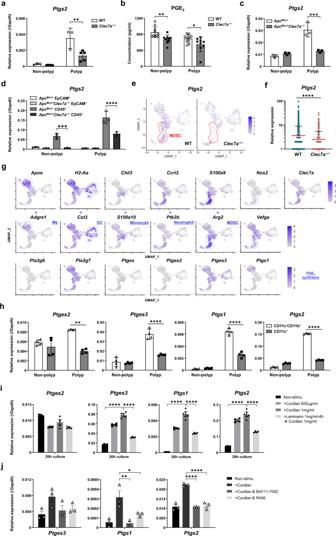Fig. 4: Dectin-1 signaling activates the expression of genes involving PGE2synthesis. a,bWT andClec7a−/−mice under SPF conditions were treated with AOM-3DSS for 16 weeks. The expression of Cox2-encodingPtgs2was determined by RT-qPCR (a, WTn= 3,Clec7a−/−n= 5; **P= 0.0030), and the concentration of PGE2in tissue homogenates was determined by ELISA (b, WTn= 10,Clec7a−/−n= 9; pooled data from 2 experiments and normalized by the protein concentration in each lysate; **P= 0.0057, *P= 0.0449).c,dThe expression ofPtgs2in intestinal polyp or non-polyp tissues (c, ***P= 0.0007), or in EpCAM+epithelial cells and in tissue-infiltrating CD45+leukocytes (d, ***P= 0.0008, ****P< 0.0001) fromApcMin/+andApcMin/+Clec7a−/−mice at 20 weeks old was determined by RT-qPCR (n= 3/group).e–gAccording to the scRNA-seq data shown in Fig.3e–h,Ptgs2expressing cells in all polyp-infiltrating myeloid cells (e) andPtgs2expression levels inPtgs2+myeloid cells (f, WTn= 1284,Clec7a−/−n= 635; ****P< 0.0001) in WT andClec7a−/−mice are shown. The expression of indicated genes including myeloid subtype-specific genes and PGE2synthase genes in WT mice are shown ing.hC57BL/6J mice were treated with AOM-3DSS for 12 weeks. CD11c+and CD11c–CD11b+cells were purified from colonic polyps and non-polyp tissues with autoMACS, and the mRNA expression of indicated genes was determined by RT-qPCR (n= 4 biologically independent samples/group; ***P= 0.0003, ****P< 0.0001).iPurified CD11b+polyp-infiltrating cells fromApcMin/+mice were harvested and were stimulated with curdlan for 20 h. Then, the expression of genes involved in PGE2synthesis was determined by RT-qPCR. Laminarin treatment was carried out for 4 h before the treatment with curdlan (n= 4 biologically independent samples/group, ****P< 0.0001).jCD11b+and CD11c+myeloid cells from colonic polyps of AOM-3DSS-treated WT mice were stimulated with curdlan (1 mg/ml) in the presence of each one of inhibitors against IκBα (BAY11-7082, 2 μM)) or SYK (R406, 2 μM). After 20 h, PGE2synthase expression was determined by qPCR (n= 3 biologically independent samples/group; *P= 0.0380, **P= 0.0037, ****P< 0.0001). Data ina,c,d,h–jare representatives of two independent experiments and are expressed as means ± SD. Data ina–d,hare analyzed using two-way ANOVA followed by Tukey’s multiple-comparisons test, infusing unpaired two-tailed Student’st-test, and ini,jusing one-way ANOVA followed by Tukey’s multiple-comparisons test. Source data are provided in the Source Data file. Statistics were computed with the PRISM v8 & v9.0 software (GraphPad Software). 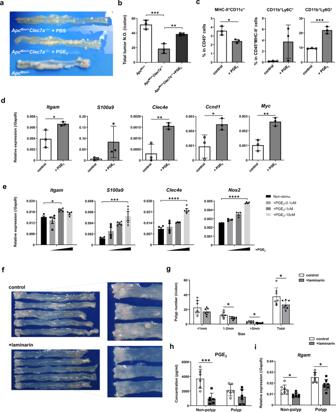Fig. 5: Oral administration of laminarin inhibits colorectal tumorigenesis, while PGE2treatment enhances tumor development. a–dApcMin/+Clec7a−/−mice (n= 3) at 8 weeks old were treated with 2% DSS for 1 week, followed by i.p. injection of PGE2(40 μg/mouse) or PBS every other day for 4 weeks. After sacrifice, colorectal polyp development was examined (a,b; ***P= 0.0006, **P= 0.0085). Populations of MHC-II+CD11c+DCs and MHC-II–CD11b+Ly6C+/Ly6G+cells in polyps were determined by flow cytometry (c; *P= 0.0193, ***P= 0.0009). Expression of indicated genes in colonic polyps was examined by RT-qPCR (d; inItgampanel, *P= 0.0463; inClec4epanel, **P= 0.0084; inCcnd1panel, *P= 0.0414; inMycpanel, **P= 0.0043) (n= 3/group).eTumor-infiltrating cells fromApcMin/+mice (n= 2) were collected and they were pooled. Then, cells were stimulated with PGE2for 20 h, and indicated gene expression was determined by RT-qPCR. Data are the means ± SD of 3–4 wells (*P= 0.0463, ***P= 0.0010, ****P< 0.0001).f–iC57BL/6J mice were administrated with AOM and were treated with 5% laminarin-containing powder food for 10 days each from 3 days before the start of DSS-treatment for 3 cycles. On week 11 after AOM injection, mice were sacrificed and the gross histology of the colon (f) and colorectal polyp number of indicated size (g; 1–2 mm, *P= 0.030; >2 mm, *P= 0.0334; Total, *P= 0.0452) were examined. The concentration of PGE2in tissue homogenate was determined by ELISA (h, normalized by protein concentration of each lysate; ***P= 0.0006), and mRNA expression ofItgam(CD11b) was examined by RT-qPCR (i; Non-polyp, *P= 0.0174; Polyp, *P = 0.0211) (n= 7/group). Data ina–d,f–iare representatives of two, and ineare representatives of three independent experiments. Data inb–e,g–iare expressed as means ± SD. Data inb,eare analyzed using one-way ANOVA followed by Tukey’s multiple-comparisons test, inc,d,gusing unpaired two-tailed Student’st-test, and inh,iusing two-way ANOVA followed by Tukey’s multiple-comparisons test. Source data are provided in the Source Data file. 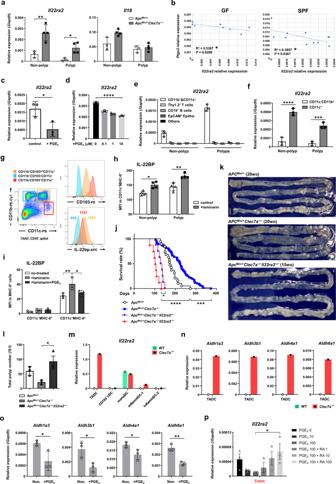Fig. 6:Il22ra2expression is highly enhanced inClec7a−/−mice and deficiency ofIl22ra2aggravates intestinal tumor development inApcMin/+Clec7a−/−mice. aApcMin/+andApcMin/+Clec7a−/−mice were sacrificed at 20 weeks old, and expression levels ofIl22ra2andIl18in intestinal polyps and non-polyp tissues were determined by RT-qPCR (ApcMin/+n= 3;ApcMin/+Clec7a−/−n= 4; **P= 0.0078, *P= 0.0148).bCorrelations betweenIl22ra2andPtgs2expression levels in colorectal polyps from GF or SPF mice after treatment with AOM-3DSS are shown (n= 8/GF,n= 11/SPF group).cIn the experiment described in Fig.5a–d, expression ofIl22ra2in colonic polyps was examined by RT-qPCR after PGE2in vivo treatment (n= 3/group, *P= 0.0261).dTumor-infiltrating cells pooled fromApcMin/+mice were harvested and were stimulated with PGE2for 20 h, followed by the measurement ofIl22ra2expression by RT-qPCR (n= 3 biologically independent samples/group; ****P< 0.0001).eClec7a−/−mice were treated with AOM-3DSS and were sacrificed after 12 weeks of AOM administration. Indicated types of cells in polyps and non-polyp tissues were purified with autoMACS andIl22ra2expression was examined by RT-qPCR (n= 3 biologically independent samples/group).fCD11c+cells and CD11c–CD11b+cells were purified with autoMACS, andIl22ra2expression in these subsets was examined by RT-qPCR (n= 3 biologically independent samples/group; ****P< 0.0001, ***P= 0.0007).gPolyp-infiltrating cells were prepared fromApcMin/+mice, and intracellular IL-22BP expression was examined in three indicated myeloid-cell populations by flow-cytometry. Colored numbers in IL-22BP panel represent mean fluorescence intensity.hThe experiment described in Fig.5fwas carried out, and 16 weeks after the AOM-DSS-treatment, mean fluorescence intensity (MFI) of IL-22BP expression in MHC-II+CD11c+DCs in colorectal polyp and non-polyp tissues was determined by flow cytometry (n= 4/group; *P= 0.0121, **P= 0.0016).iWT mice were administrated with 5% laminarin in diet from 3 days before 1.5% DSS treatment and continued for 7 days until the end of DSS treatment. During DSS-treatment, mice were also i.p. injected with PGE2every other day for 4 times. One day after the last PGE2injection, mice were sacrificed and MFI of IL-22BP expression in MHC-II+CD11c+DCs was determined by flow cytometry (n= 3/group; **P= 0.0035, *P= 0.02323).jSurvival rates of indicated mice are shown (ApcMin/+n= 19;ApcMin/+Clec7a−/−n= 66;ApcMin/+Clec7a−/−Il22ra2+/−n= 8;ApcMin/+Clec7a−/−Il22ra2−/−n= 8; ****P< 0.0001, ***P= 0.0003, *P= 0.0179).kRepresentative pictures of the small intestine ofApcMin/+andApcMin/+Clec7a−/−mouse of 20 weeks old andApcMin/+Clec7a−/−Il22ra2−/−mouse of 15 weeks old are shown.lTotal polyp number in the intestine ofApcMin/+(n= 3),ApcMin/+Clec7a−/−(n= 3), andApcMin/+Clec7a−/−Il22ra2−/−(n= 3) mice are shown (*P= 0.0125).mIn the scRNA-seq analysis described in Fig.3e–h, the expression levels ofIl22ra2were determined in each colorectal polyp-infiltrating DC subset.nAs inm, RA synthase expression levels in TADC from WT andClec7a−/−mice were determined by scRNA-seq.oCD11b+and CD11c+cells isolated from WT mouse colon were treated with 10 μM PGE2for 20 h, and expression levels of genes encoding RA synthases were examined by RT-qPCR (n= 3 biologically independent samples/group;Aldh1a3, *P= 0.0340;Aldh3b1, *P= 0.0261;Aldh4a1, *P= 0.0472;Aldh6a1, **P= 0.0023).pCD11b+and CD11c+cells isolated from WT mouse colon were treated with indicated doses of PGE2(μM) and RA (μM) for 20 h, and expression level ofIl22ra2was examined by RT-qPCR (n= 3 biologically independent samples/group; *P= 0.030). Data ina,c–l,o,pare representatives of two independent experiments, and ina,c,d–f,h,i,l,o,pare expressed as means ± SD. Data ina,f,h,iare analyzed using two-way ANOVA followed by Tukey’s multiple-comparisons test, inbusing Pearson’s correlation coefficient (r) test, inc,ousing two-tailed Student’st-test, ind,l,pusing one-way ANOVA followed by Tukey’s multiple-comparisons test and injusing Mantel-Cox log-rank test. Source data are provided in the Source Data file. 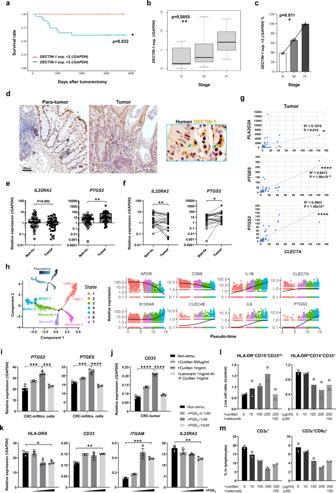Fig. 7: The expressions of PGE2-synthesizing enzymes andIL22RA2are modified in CRC patients. a–cSpecimens from 36 CRC patients were collected and the post-surgery survival rates of the patients withCLEC7AmRNA expression <2 (n= 12) or >2 (2–20) (n= 24) (normalized byGAPDH) in tumor tissues are shown (a). The correlation betweenCLEC7Aexpression levels and tumor TNM stage (b,n= 13 in Stage II,n= 12 in Stage III,n= 8 in Stage IV), and the correlation between the proportion of patients withCLEC7Aexpression >2 in each stage (c,n= 13 in Stage II,n= 12 in Stage III, n = 8 in Stage IV) are shown. Tumor TNM stage was determined according to the individual clinical information. In boxplot (b), the central horizontal line shows the median; the upper and lower bounds of box show third and first quartile; the upper and lower horizontal lines show the maxima and minima of the data.dImmunohistochemical staining of human Dectin-1 in tumor and non-tumor colon tissues in CRC patients. Green arrows show Dectin-1+cells. Representative photos from two independent experiments containing nine samples of eight patients are shown.eSpecimens from total 68 CRC patients were collected including 23 pairs of tumors and non-tumor specimens from the same individuals.IL22RA2andPTGS2expression in tumors and non-tumor tissues were examined by RT-qPCR (n= 47 in tumor group,n= 44 in non-tumor group; **P= 0.0084).fTwenty-three pairs of tumor and non-tumor specimens from the same individual were collected, andIL22RA2andPTGS2expression were examined (n= 23/group; **P= 0.0067, *P= 0.0179).gCorrelations of the expression (normalized byGAPDH) between PGE2synthesizing enzymes andCLEC7Ain CRC tissues (n= 47/group).hPseudotime/trajectory analysis was carried out by using a scRNA-seq dataset (GSE178318) of CRC-infiltrating myeloid cells, in which fully differentiated DCs were excluded. Cell states and their annotations (left panel), and kinetics of relative expression levels of MDSC and macrophage-associated gene markers along the MDSC ‘differentiation’ pseudo-time (right panels) are shown. TAM: tumor-associated macrophage; Mono-DC: monocyte-derived DC.i,jTumor and non-tumor tissue-infiltrating cells were collected from CRC patients and were stimulated with curdlan for 20 h. In the case of laminarin treatment, cells were first treated with laminarin for 4 h, then curdlan was added to the culture. Expression of PGE2synthesizing enzymes (i;PTGS2, 1st ***P= 0.0001, 2nd ***P= 0.0004;PTGES, ***P= 0.0001, ****P< 0.0001) and CD33 (j; ****P< 0.0001) was determined by RT-qPCR. Data are the means ± SD of 3 wells.kTumors from CRC patients were collected and after mincing, small pieces were cultured in the presence of PGE2for 20 h. The expression of indicated genes was determined by RT-qPCR. Data are the means ± SD of 3 wells (HLA-DRA, *P= 0.0122;CD33, **P= 0.0033;ITGAM, ***P= 0.0004;IL22RA2, **P= 0.0018).lHuman PBMCs were harvested from healthy volunteers and were treated with curdlan and celecoxib at the indicated doses in the presence of rGM-CSF + IL-6. After the culture for 5 days, indicated cell number was determined by flow cytometry and was normalized with the average number in control (curdlan 0) group.mIn the experiment described inl, after the culture, proportions of whole T cells and CD8+T cells were determined by flow cytometry. Data ini–kare representatives of three, and inl,mare representatives of two independent experiments and are expressed as means ± SD. Data inaare analyzed using Mantel-Cox log-rank test, inb,cusing Spearman rank correlation test, ineusing two-tailed Student’st-test, infusing Wilcoxon matched-pairs signed rank test, ingusing Pearson’s correlation coefficient (r) test, and ini,j,kusing one-way ANOVA followed by Tukey’s multiple-comparisons test. Source data are provided in the Source Data file. For CRC patient study, categorical variables were compared by the Fisher tests, correlation was analyzed by the Spearman’s correlation test and statistical analysis was performed using the R software (version 4.0.3, R Foundation). Difference of P -value < 0.05 were considered statistically significant. Reporting summary Further information on research design is available in the Nature Portfolio Reporting Summary linked to this article.